Retromer deficiency in Tauopathy models enhances the truncation and toxicity of Tau 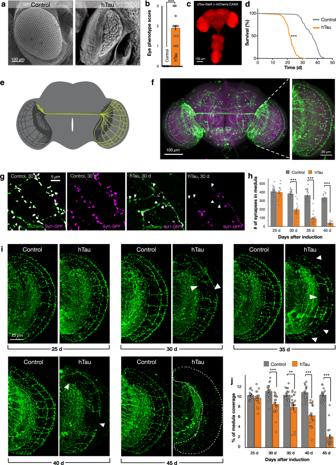Fig. 1: Expression of human Tau disrupts eye development, reduces adult lifespan, and induces synapse loss and axonal retraction. aExamples of eyes from control [GMR-Gal4, UAS-mCD8GFP] versus hTau expressing animals [GMR-Gal4, UAS-hTau, UAS-ControlRi].bEye disruption scores for indicated genotypes. Data are presented as mean values +/− SEM.cDrosophilaadult brain expression ofdTau-Gal4 labeled with UAS-mCherry-CAAX.dSurvival analyses of control animals [dTau-Gal4, UAS-mCD8GFP,tubulin-Gal80ts] and hTau expressing adults [dTau-Gal4, UAS-hTau,tubulin-Gal80ts]eSchematic of the contralaterally projecting DC neurons subset of theato-Gal4 line.fato-Gal4 expressing neurons in adultDrosophilabrain (left) with magnification of DC axonal subset in the medulla (right).gDC neuron medulla synapses labeled by Synaptotagmin-GFP [magenta] in control [ato-Gal4, UAS-Syt1-GFP, UAS-mCherry, UAS-mCD8GFP,tubulin-Gal80ts] and hTau expressing [ato-Gal4, UAS-hTau, UAS-Syt1-GFP, UAS-mCherry,tubulin-Gal80ts] animals, at 30 days after induction of transgene expression. In the control, axonal varicosities (mCherry) coincide with Syt1 labeling, in hTau expressing neurons many axonal varicosities lack Syt1 (arrowheads).hQuantification of the number of medulla synapses labeled by Synaptotagmin-GFP in control [ato-Gal4, UAS-Syt1-GFP, UAS-mCherry, UAS-mCD8GFP,tubulin-Gal80ts] and hTau [ato-Gal4, UAS-hTau, UAS-Syt1-GFP, UAS-mCherry,tubulin-Gal80ts] expressing animals in increments from 25 to 40 days after induction of transgene expression. Data are presented as mean values +/− SEM.iDC neuron axons in hTau [ato-Gal4, UAS-hTau, UAS-mCherry,tubulin-Gal80ts] and control animals [ato-Gal4, UAS-mCherry, UAS-mCD8GFP,tubulin-Gal80ts] from 25 to 45 days after induction of transgene expression. Gaps in axonal structure induced by hTau expression are indicated with arrowheads, when <4% axons are present, the medulla is outlined with dashed lines.jQuantification of medulla area occupied by DC neuron axons in hTau [ato-Gal4, UAS-hTau, UAS-mCherry,tubulin-Gal80ts] and control animals [ato-Gal4, UAS-mCD8GFP, UAS-mCherry,tubulin-Gal80ts]. Data are presented as mean values +/− SEM. Mann–Whitney test, ***p< 0.001 for eye disruption scores comparison between control (n= 32) and hTau (n= 34) (b). Mantel-Cox test, ***p< 0.001 for survival analysis of control (n= 202) vs. hTau (n= 192) (d), Mann–Whitney test,p= 0.701 for control (n= 18) vs. hTau (n= 15) (h, 25 days post induction), ***p< 0.001 for control (n= 18) vs. hTau (n= 16) (h, 30 days post induction), ***p< 0.001 for control (n= 17) vs. hTau (n= 19) (h, 35 days post induction), ***p< 0.001 for control (n= 16) vs. hTau (n= 15) (h, 40 days post induction). Mann–Whitney test,p= 0.1427 for control (n= 18) vs. hTau (n= 18) (j, 25 days post induction), ***p< 0.001 for control (n= 20) vs. hTau (n= 20) (j, 30 days post induction), **p= 0.0022 for control (n= 17) vs. hTau (n= 20) (j, 35 days post induction), ***p< 0.001 for control (n= 18) vs. hTau (n= 20) (j, 40 days post induction), ***p< 0.001 for control (n= 19) vs. hTau (n= 20) (j, 45 days post induction).nindicates independent biological replicates. Source data are provided as a Source Data file. Alteration of the levels, localization or post-translational processing of the microtubule associated protein Tau is associated with many neurodegenerative disorders. Here we develop adult-onset models for human Tau (hTau) toxicity in Drosophila that enable age-dependent quantitative measurement of central nervous system synapse loss and axonal degeneration, in addition to effects upon lifespan, to facilitate evaluation of factors that may contribute to Tau-dependent neurodegeneration. Using these models, we interrogate the interaction of hTau with the retromer complex, an evolutionarily conserved cargo-sorting protein assembly, whose reduced activity has been associated with both Parkinson’s and late onset Alzheimer’s disease. We reveal that reduction of retromer activity induces a potent enhancement of hTau toxicity upon synapse loss, axon retraction and lifespan through a specific increase in the production of a C-terminal truncated isoform of hTau. Our data establish a molecular and subcellular mechanism necessary and sufficient for the depletion of retromer activity to exacerbate Tau-dependent neurodegeneration. Tau, a microtubule-associated protein, stabilizes microtubule structures [1] and is abundant in neural tissues [2] , [3] , predominantly within the axonal tracts of neurons [4] . Misfolded Tau species can contribute to insoluble aggregates that deposit within neurons in a class of neuropathologies known as Tauopathies [5] . Post-translational modified forms of Tau including hyperphosphorylation, as well as N- and C-terminal truncation, have been established as constituents of these pathological Tau deposits [6] and these post-translational alterations can enhance both Tau tangle formation and fibrilogenicity [7] , [8] . A multitude of intracellular trafficking pathways are involved in the resolution and degradation of Tau aggregates [9] , [10] , [11] and dysfunction of these pathways can exacerbate Tau accumulation and toxicity [12] . The retromer complex is an evolutionarily conserved protein assembly that plays an essential role in the retrograde transport of proteins and associated lipids from endosomes to the trans-Golgi network and in the recycling of this cargo from endosomes back to the cell surface. The complex consists of a heterotrimeric protein core comprised of VPS26, VPS29, and VPS35 [13] , [14] , [15] , [16] . This core assembly can interact with a variety of other intracellular trafficking proteins to regulate the transport of a wide range of cargo that enter the endosomal network either from the plasma membrane, via the biosynthetic or autophagic pathways, or from other sources. Mutations in retromer components are associated with familial Parkinson’s disease (PD) [17] , [18] , [19] , [20] , [21] , [22] and defects in retromer activity are also linked with Alzheimer’s disease (AD) [23] , [24] . Consistent with an association of retromer with Alzheimer’s disease, retromer activity is reduced in the entorhinal cortex of late onset AD patients [25] . Decreasing retromer activity can inhibit long-term potentiation at hippocampal synapses [26] and exacerbates memory deficits in a rodent AD model [27] . The molecular mechanisms through which retromer depletion may contribute to AD are still not fully understood. Retromer deficiency can alter Amyloid Beta (Aβ) levels [25] , [28] , [29] and rodents deficient in retromer activity have increased levels of some species of Tau in the cerebrospinal fluid (CSF) [24] , similar to observations of Tau in the CSF of AD patients [24] , [30] , [31] . Here, we have investigated the molecular and cellular mechanisms of the interaction of retromer with human Tau (hTau), using both in vivo Drosophila models and cell models of Tau toxicity. We find that reduction of retromer activity induces a potent enhancement of hTau toxicity through a specific and singular increase in the production of a C-terminal truncated isoform of hTau. We further demonstrate that interaction of the retromer complex with the late endosome protein Rab7 is critical for the enhancement of Tau-dependent neurodegeneration. Our data establish a molecular and cellular rationale causally linking deficient retromer activity with enhanced Tau toxicity. Expression of human Tau can disrupt development, reduce adult lifespan and induce axon retraction To begin to investigate the effects in Drosophila of expression of human Tau, we expressed a transgenic wildtype (WT) (2N4R) variant of hTau in the Drosophila eye [32] . As described previously [33] , expression of hTau during eye development induces aberrant morphology compared to controls which can be assigned a quantitative score (Fig. 1a, b and Supplementary Fig. 1a ). Using these scoring criteria, eye morphology in hTau-expressing animals scored on average 1.89 AU ( p < 0.001) compared to controls (0.04) (Fig. 1b ), consistent with previous studies of hTau expression during development. Fig. 1: Expression of human Tau disrupts eye development, reduces adult lifespan, and induces synapse loss and axonal retraction. a Examples of eyes from control [GMR-Gal4, UAS-mCD8GFP] versus hTau expressing animals [GMR-Gal4, UAS-hTau, UAS-Control Ri ]. b Eye disruption scores for indicated genotypes. Data are presented as mean values +/− SEM. c Drosophila adult brain expression of dTau -Gal4 labeled with UAS-mCherry-CAAX. d Survival analyses of control animals [ dTau -Gal4, UAS-mCD8GFP, tubulin -Gal80 ts ] and hTau expressing adults [ dTau -Gal4, UAS-hTau, tubulin -Gal80 ts ] e Schematic of the contralaterally projecting DC neurons subset of the ato -Gal4 line. f ato -Gal4 expressing neurons in adult Drosophila brain (left) with magnification of DC axonal subset in the medulla (right). g DC neuron medulla synapses labeled by Synaptotagmin-GFP [magenta] in control [ ato -Gal4, UAS-Syt1-GFP, UAS-mCherry, UAS-mCD8GFP, tubulin -Gal80 ts ] and hTau expressing [ ato -Gal4, UAS-hTau, UAS-Syt1-GFP, UAS-mCherry, tubulin -Gal80 ts ] animals, at 30 days after induction of transgene expression. In the control, axonal varicosities (mCherry) coincide with Syt1 labeling, in hTau expressing neurons many axonal varicosities lack Syt1 (arrowheads). h Quantification of the number of medulla synapses labeled by Synaptotagmin-GFP in control [ ato -Gal4, UAS-Syt1-GFP, UAS-mCherry, UAS-mCD8GFP, tubulin -Gal80 ts ] and hTau [ ato -Gal4, UAS-hTau, UAS-Syt1-GFP, UAS-mCherry, tubulin -Gal80 ts ] expressing animals in increments from 25 to 40 days after induction of transgene expression. Data are presented as mean values +/− SEM. i DC neuron axons in hTau [ ato -Gal4, UAS-hTau, UAS-mCherry, tubulin -Gal80 ts ] and control animals [ ato -Gal4, UAS-mCherry, UAS-mCD8GFP, tubulin -Gal80 ts ] from 25 to 45 days after induction of transgene expression. Gaps in axonal structure induced by hTau expression are indicated with arrowheads, when <4% axons are present, the medulla is outlined with dashed lines. j Quantification of medulla area occupied by DC neuron axons in hTau [ ato -Gal4, UAS-hTau, UAS-mCherry, tubulin -Gal80 ts ] and control animals [ ato -Gal4, UAS-mCD8GFP, UAS-mCherry, tubulin -Gal80 ts ]. Data are presented as mean values +/− SEM. Mann–Whitney test, *** p < 0.001 for eye disruption scores comparison between control ( n = 32) and hTau ( n = 34) ( b ). Mantel-Cox test, *** p < 0.001 for survival analysis of control ( n = 202) vs. hTau ( n = 192) ( d ), Mann–Whitney test, p = 0.701 for control ( n = 18) vs. hTau ( n = 15) ( h , 25 days post induction), *** p < 0.001 for control ( n = 18) vs. hTau ( n = 16) ( h , 30 days post induction), *** p < 0.001 for control ( n = 17) vs. hTau ( n = 19) ( h , 35 days post induction), *** p < 0.001 for control ( n = 16) vs. hTau ( n = 15) ( h , 40 days post induction). Mann–Whitney test, p = 0.1427 for control ( n = 18) vs. hTau ( n = 18) ( j , 25 days post induction), *** p < 0.001 for control ( n = 20) vs. hTau ( n = 20) ( j , 30 days post induction), ** p = 0.0022 for control ( n = 17) vs. hTau ( n = 20) ( j , 35 days post induction), *** p < 0.001 for control ( n = 18) vs. hTau ( n = 20) ( j , 40 days post induction), *** p < 0.001 for control ( n = 19) vs. hTau ( n = 20) ( j , 45 days post induction). n indicates independent biological replicates. Source data are provided as a Source Data file. Full size image Having established expression of our hTau reagents could recapitulate prior observations during development, we next sought to determine the effects of hTau expression in adult animals in a physiologically appropriate pattern. To do this, we generated a Gal4 insertion in the endogenous Drosophila Tau ( dTau ) gene and coupled this with temporal control of expression only in adults [34] . We did note that dTau mRNA expression was reduced in this line relative to controls (Supplementary Fig. 1b ), however even null mutants of dTau do not alter animal lifespan [35] . We confirmed using a reporter that dTau -Gal4 has broad neural expression in adult Drosophila similar to dTau protein expression [36] (Fig. 1c ). Using this line, we then expressed hTau only in adulthood using temperature-controlled induction beginning 3 days after adult emergence (eclosion). Compared to GFP expressing control animals, which had a median survival age of 37 days, we found animals expressing in hTau in adulthood had a 40.5% reduction ( p < 0.001) in median survival to 22 days (Fig. 1d ). Thus, expression of human Tau in adult Drosophila within the pattern of dTau expression dramatically reduces lifespan. In numerous paradigms, increased levels of Tau result in the retraction and degeneration of axons [37] , but this is difficult to assay when expression patterns are broad, such as in dTau -Gal4. We therefore sought to develop an assay that would allow us to image with single axon resolution the effects of hTau expression on adult Drosophila neurons in vivo. To do this, we expressed hTau in a subset of adult neurons labeled by the ato -Gal4 line [38] again using temperature-controlled induction to ensure expression only in adults. Neurons labeled by this line include a group of ~39 neurons [39] , designated Dorsal Cluster (DC) neurons, of which ~11 project contralateral axons to make stereotypical sparse synaptic connections forming a lattice in the optic medulla (Fig. 1e, f ). This sparse and reproducible distribution allowed us to image individual axons and synapses in this brain region. We first examined the synapses produced by DC neurons, labeled with Synaptotagmin-GFP (Fig. 1g ), in control animals as they aged. We found that the number of DC neuron synapses was unchanged until 25 days after eclosion in control animals (Fig. 1h ). After this age, there was a modest continual decrease in the number of DC neuron synapses such that 40-day old animals had on average 18% less ( p < 0.001) synapses compared to 25-day old control animals (Fig. 1h ). We then expressed hTau in these neurons beginning 3 days after adult eclosion. Similar to control animals, we observed no change in the number of DC neuron synapses during the first 25 days of hTau expression. However, after this age, we observed a rapid loss of DC neuron medulla synapses in hTau expressing animals (Fig. 1g, h ) with a 49% ( p < 0.001) decrease in synapse numbers at 30 days, a 75% ( p < 0.001) decrease after 35 days and an 89% ( p < 0.001) decrease after 40 days compared to control animals of the same age. Therefore, expression of hTau in adult DC neurons results in a progressive loss of synaptic connections. We next examined if this loss of synapses was accompanied by changes in axons of DC neurons in the medulla during adult lifespan. Unlike DC neuron synapses, we found no change in the area occupied by DC neuron axons within the medulla through lifespan in control animals (Fig. 1i, j ). When hTau was expressed in DC neurons, we also observed no change in the medulla area occupied by these axons for the first 25 days after hTau expression (Fig. 1i, j ). However, beginning at 30 days, the axons in hTau expressing animals became obviously perturbed with noticeable axonal loss (Fig. 1i, j ) evidenced by a 23% ( p < 0.001) reduction in DC neuron medulla axonal area compared to controls. Axonal loss was coincident with the thinning and fragmentation of the remaining axons (Supplementary Fig. 1c ). Progressively more DC neuron axons were lost in hTau expressing animals as they continued to age (Fig. 1i, j ), until only 20% ( p < 0.001) of DC medulla axons were present compared to controls at 45 days after the induction of hTau expression. The retraction and loss of DC neuron axons was not accompanied by cell death of DC neurons however, as the number of DC neurons in hTau expressing animals did not decline compared to controls at any age timepoint (Supplementary Fig. 1d – f ). To determine if axons of DC neurons were also perturbed when hTau was broadly expressed, we labeled DC neurons with ato -lexA [39] while simultaneously expressing hTau with dTau -Gal4. We also observed a loss of DC neuron axons in the context of broad hTau expression (Supplementary Fig. 1g ), similar to that seen when hTau was expressed with ato -Gal4, consistent with axon loss as a recurrent outcome of hTau expression in neurons. In summary, expression of human Tau in Drosophila adults reduces lifespan and induces an age-dependent progressive loss of synapses and retraction of axons. Inhibition of retromer enhances the toxicity of human Tau We next sought to examine the effects of inhibiting retromer components on hTau-mediated toxicity in each of the Tau models described above. We decided to employ transgenic RNAi ( Ri ) constructs to allow tissue-specific knockdown of VPS26, VPS29, and VPS35 proteins. We first validated the efficiency of these constructs to reduce retromer protein levels (Supplementary Fig. 2a, b ). We observed an 86% reduction of VPS26 ( p < 0.001), an apparently complete inhibition of VPS29 expression ( p < 0.001), and a 41% reduction of VPS35 ( p < 0.02) using these lines. We next assessed the effects of knock-down using these lines upon eye morphology. We found that consistent with previous reports [40] , [41] , inhibition of retromer components did not induce aberrant eye development (Fig. 2b and Supplementary Fig. 2c ). We then combined inhibition of retromer with these constructs together with simultaneous expression of human Tau. When hTau was expressed while VPS26, VPS29, or VPS35 were inhibited, we found a significant increase of the disruption of eye morphology compared to hTau expression alone (Fig. 2a, b ) (+37% [ p < 0.001] hTau & Vps26 Ri vs hTau, +41% [ p < 0.001] hTau & Vps29 Ri vs hTau, and +24% [ p < 0.003] hTau & Vps35 Ri vs hTau). The magnitude of the enhancement we observed was consistent with the relative efficiency of RNAi inhibition (Supplementary Fig. 2a, b ). These results suggested that reduction of retromer activity could enhance the toxicity of Tau at least during eye development. Fig. 2: Retromer depletion exacerbates the toxicity of human Tau. a Eye morphology in control [GMR-Gal4, UAS-mCD8GFP], hTau expression together with control RNAi [GMR-Gal4, UAS-hTau, UAS-GFP Ri ] and hTau expression [GMR-Gal4, UAS-hTau] together with RNAi inhibition of retromer components (plus UAS-Vps35 Ri or UAS-Vps29 Ri or UAS-Vps26 Ri ]. b Eye disruption scores for indicated genotypes. Data are presented as mean values +/− SEM. c Survival analyses of hTau [ dTau -Gal4, UAS-hTau, UAS-Cherry Ri , tubulin -Gal80 ts ] and hTau expressing adults [ dTau -Gal4, UAS-hTau, tubulin -Gal80 ts ] together with retromer inhibition [plus UAS-Vps35 Ri or UAS-Vps29 Ri or UAS-Vps26 Ri ]. d DC neuron medulla axons with hTau expression alone [ ato -Gal4, UAS-hTau, UAS-mCherry, UAS-mCD8GFP, tubulin -Gal80 ts ] and hTau expression [ ato -Gal4, UAS-hTau, UAS-mCherry, tubulin -Gal80 ts ] together with retromer inhibition [UAS-Vps35 Ri or UAS-Vps29 Ri or UAS-Vps26 Ri ] from 25 to 45 days after onset of transgene expression. Gaps in axonal structure induced by hTau expression are indicated with arrowheads, when <4% axons are present, the medulla is outlined with dashed lines. e Quantification of medulla area occupied by DC neuron axons with hTau expression alone [ ato -Gal4, UAS-hTau, UAS-mCherry, UAS-mCD8GFP, tubulin -Gal80 ts ] and hTau expression [ ato -Gal4, UAS-hTau, UAS-mCherry, tubulin -Gal80 ts ] together with retromer inhibition [UAS-Vps35 Ri or UAS-Vps29 Ri or UAS-Vps26 Ri ] from 25 to 45 days after onset of transgene expression. Data are presented as mean values +/− SEM. Kruskal–Wallis test, *** p < 0.001, for eye disruption scores across all genotypes with multiple comparisons between hTau ( n = 34) and hTau plus Vps35 Ri ( n = 38) (Dunnett’s test ** p = 0.003), hTau and hTau plus Vps29 Ri ( n = 38) (Dunnett’s test *** p < 0.001), and hTau and hTau plus Vps26 Ri ( n = 29) (Dunnett’s test *** p < 0.001). n = 23 for control, n = 31 for Vps35 Ri , n = 30 for Vps29 Ri and n = 31 for Vps26 Ri ( b ). Mantel-Cox test, *** p = 0.0005 for survival analysis of hTau ( n = 148) vs. hTau plus Vps35 Ri ( n = 153), *** p < 0.001 for hTau vs. hTau plus Vps29 Ri ( n = 126), and *** p < 0.001 for hTau vs. hTau plus Vps26 Ri ( n = 173) ( c ). Kruskal-Wallis test, p = 0.4212 ( e , 25 days post induction) for hTau ( n = 21) vs. hTau plus Vps35 Ri ( n = 20) (Dunnett’s test p = 0.9855), hTau vs. hTau plus Vps29 Ri ( n = 24) (Dunnett’s test p = 0.9999), hTau vs. hTau plus Vps26 Ri ( n = 18) (Dunnett’s test p = 0.2582), n = 18 for control. Kruskal-Wallis test, * p = 0.0351 ( e , 30 days post induction) for hTau ( n = 20) vs. hTau plus Vps35 Ri ( n = 19) (Dunnett’s test p = 0.9974), hTau vs. hTau plus Vps29 Ri ( n = 20) (Dunnett’s test p = 0.988), hTau vs. hTau plus Vps26 Ri ( n = 20) (Dunnett’s test * p = 0.0476), n = 20 for control. Kruskal–Wallis test, *** p < 0.001 ( e , 35 days post induction) for hTau ( n = 20) vs. hTau plus Vps35 Ri ( n = 20) (Dunnett’s test p = 0.6797), hTau vs. hTau plus Vps29 Ri ( n = 20) (Dunnett’s test ** p = 0.0091), and hTau vs. hTau plus Vps26 Ri ( n = 22) (Dunnett’s test *** p < 0.001), n = 17 for control. Kruskal-Wallis test, *** p < 0.001 ( e , 40 days post induction) for hTau ( n = 20) vs. hTau plus Vps35 Ri ( n = 22) (Dunnett’s test *** p < 0.001), hTau vs. hTau plus Vps29 Ri ( n = 20) (Dunnett’s test *** p = 0.0005), and hTau vs. hTau plus Vps26 Ri ( n = 15) (Dunnett’s test *** p < 0.001), n = 18 for control. Kruskal–Wallis test, p = 0.2815 ( e , 45 days post induction) for hTau ( n = 20) vs. hTau plus Vps35 Ri ( n = 11) (Dunnett’s test p = 0.1407), hTau vs. hTau plus Vps29 Ri ( n = 19) (Dunnett’s test p < 0.1209), and hTau vs. hTau plus Vps26 Ri ( n = 11) (Dunnett’s test p = 0.1728), n = 19 for control. n indicates independent biological replicates. Source data are provided as a Source Data file. Full size image To determine if this interaction also occurred in adult neurons, we next inhibited retromer components while co-expressing hTau. We first examined the effects of retromer inhibition alone upon lifespan when expressed using dTau -Gal4. We observed that inhibition of VPS29 did not significantly alter median lifespan (36 days Vps29 Ri vs 37 days control Ri , [ p = 0.8]), however, inhibition of VPS26 did significantly reduce median lifespan by 5.4% ( p < 0.001, 35 days Vps26 Ri vs 37 days control Ri ), while VPS35 inhibition reduced median lifespan by 19% ( p < 0.001, 30 days Vps35 Ri vs 37 days control Ri ) (Supplementary Fig. 2d ). We then co-expressed these constructs together with hTau in adults. We found that inhibition of retromer components further reduced median survival compared to hTau expression alone (Fig. 2c ), with VPS26 inhibition reducing lifespan by an additional 27% ( p < 0.001, 16 days hTau & Vps26 Ri vs hTau 22 days), VPS29 inhibition reducing lifespan by an additional 23% ( p < 0.001, 17 days hTau & Vps29 Ri vs hTau 22 days), and VPS35 inhibition reducing median lifespan by a further 9% ( p < 0.001, 20 days hTau & Vps35 Ri vs hTau 22 days). Since VPS35 inhibition alone can significantly alter median lifespan, it is difficult to conclude if the combination with hTau is additionally more detrimental in this assay, however, the pronounced effect of VPS29 inhibition (which does not alter lifespan in controls), and VPS26 inhibition (which reduces lifespan fivefold more in the presence of hTau than in controls) was consistent with an enhancement of hTau toxicity when retromer activity is inhibited. Building upon this finding, we then examined the effects of retromer depletion upon hTau-dependent axonal retraction in adult neurons. We found no alteration of the area occupied by DC neuron axons within the medulla when VPS26, VPS29, or VPS35 were inhibited alone in these neurons throughout lifespan (Supplementary Fig. 2e ). We then coupled retromer inhibition with expression of hTau in DC neurons. While axonal retraction did not initiate at an earlier timepoint, we did observe a significant enhancement of axon loss (Fig. 2d, e ) in these animals beginning 35 days of age. Inhibition of VPS26 increased axon loss by +15% ( p < 0.047, hTau & Vps26 Ri vs hTau) at 30 days, though inhibition of VPS35 and VPS29 did not significantly increase axonal loss at this age. Inhibition of VPS26 increased axon loss by 41% ( p < 0.001, hTau & Vps26 Ri vs hTau) and inhibition of VPS29 by +16% ( p < 0.01, hTau & Vps29 Ri vs hTau) at 35 days though inhibition of VPS35 did not significantly increase axonal loss at this age. However, by 40 days, inhibition of VPS35 did significantly increase axonal loss by 43% ( p < 0.001, hTau & Vps35 Ri vs hTau) as continually did inhibition of VPS26 (+56.7%, p < 0.001) and VPS29 (+35%, p < 0.001). This axonal loss progressed to 45 days such that only 12.1% ( p < 0.001) of axons were retained on average when any component of the retromer complex was inhibited compared to controls (Fig. 2d, e ). Therefore, as with eye morphology and longevity, retromer inhibition also enhanced the retraction of axons in response to the expression of human Tau. We also questioned if oppositely increasing retromer expression could modulate Tau-dependent axonal degeneration. However, we found that increasing the expression of Vps26, Vps29 or Vps35 alone in DC neurons using transgenes induced considerable axonal loss (Supplementary Fig. 2f ) precluding additional interaction experiments. It is noteworthy that increased expression of retromer components also induces neurodegeneration in mice [42] . In summary, depletion of retromer activity, which does not compromise axonal integrity alone, does exacerbate the Tau-dependent neurotoxicity. Retromer inhibition increases Tau truncation We next sought to interrogate potential mechanisms through which retromer depletion could increase the toxicity of Tau. Alteration of the phosphorylation status of Tau has been linked to increased toxicity [43] , [44] so we first compared the phosphorylation status of hTau in vivo using the phosphospecific antibodies PHF-1, AT8, and AT100 [45] when hTau was expressed alone or when retromer activity was simultaneously reduced. However, we found no change in the phosphorylation state of Tau when retromer activity was depleted as compared to hTau expression alone with these reagents (Fig. 3a, b ). Truncated isoforms of Tau have become increasingly appreciated as important pathogenic contributors to Tau toxicity [7] , [8] , [46] , [47] , [48] , [49] . We therefore probed for truncated Tau using an antibody specific to hTau truncated at Aspartate 421 [hTau 421D ] [46] . In stark contrast to measurements of Tau phosphorylation, we observed a dramatic 4.2-fold increase ( p < 0.001) in the levels of hTau 421D when VPS26 was inhibited together with hTau expression (Fig. 3a, b ). This increase was also observed when VSP29 (3.4-fold [ p < 0.001], hTau & Vps29 Ri vs hTau) or VPS35 (2.0-fold [ p < 0.05], hTau & Vps35 Ri vs hTau) were inhibited when compared to hTau expression alone (Fig. 3a, b ). Fig. 3: Human Tau truncation requires the caspase Dronc. a hTau protein analyses from head lysates of controls [GMR-Gal4, UAS-mCD8GFP], hTau expressing animals [GMR-Gal4, UAS-hTau, UAS-GFP Ri ], and hTau [GMR-Gal4, UAS-hTau] expression together with retromer inhibition [UAS-Vps35 Ri or UAS-Vps29 Ri or UAS-Vps26 Ri ]. b Quantification of total Tau protein levels, Tau phosphorylation (PHF-1, AT8, and AT100) or truncation (Tau 421D ). Data are presented as mean values +/− SEM. c Protein analyses of truncated Tau levels in CN1.4 mouse cortical neurons expressing inducible full-length human Tau (0N4R) and scrambled shRNA or shRNAs against murine VPS26A, or VPS29, or VPS35. d Quantification of truncated Tau levels in CN1.4 neurons expressing human Tau and scrambled shRNA or shRNAs against murine VPS26A, or VPS29, or VPS35. Data are presented as mean values +/− SEM. e Protein analyses of head lysates from control [GMR-Gal4, UAS-mCD8GFP], hTau expressing [GMR-Gal4, UAS-hTau, UAS-GFP Ri ] animals, and hTau expression together with Dronc inhibition [GMR-Gal4, UAS-hTau, UAS-Dronc Ri ], probed with anti-hTau 421D (top) or anti-total Tau [TauC] (middle). f Quantification of total and truncated Tau levels from RNAi control [GMR-Gal4, UAS-hTau, UAS-GFP Ri ] animals and hTau expression together with Dronc inhibition [GMR-Gal4, UAS-hTau, UAS-Dronc Ri ]. Data are presented as mean values +/− SEM. g DC neuron medulla axons in control [ ato -Gal4, UAS-mCherry, UAS-mCD8GFP, tubulin -Gal80 ts ], hTau expressing [ ato -Gal4, UAS-hTau, UAS-mCherry, UAS-mCD8GFP, tubulin -Gal80 ts ] animals, and hTau expression together with Dronc inhibition [ ato -Gal4, UAS-hTau, UAS-Dronc Ri , UAS-mCherry, tubulin -Gal80 ts ] from 25 to 45 days after onset of transgene expression. h Quantification of medulla area occupied by DC neuron control [ ato -Gal4, UAS-mCherry, UAS-mCD8GFP, tubulin -Gal80 ts ], hTau expressing [ ato -Gal4, UAS-hTau, UAS-mCherry, UAS-mCD8GFP, tubulin -Gal80 ts ] animals, and hTau expression together with Dronc inhibition [ ato -Gal4, UAS-hTau, UAS-Dronc Ri , UAS-mCherry, tubulin -Gal80 ts ] from 25 to 45 days after onset of transgene expression. Data are presented as mean values +/− SEM. One-Way ANOVA, p = 0.5466, n = 3 for all genotypes ( b , total hTau), One-way ANOVA, p = 0.8216, n = 3 for all genotypes ( b , PHF-1), One-way ANOVA, p = 0.8216 n = 3 for all genotypes, ( b , PHF-1), One-way ANOVA, p = 0.8791, n = 3 for all genotypes ( b , AT8), One-Way ANOVA, p = 0.8982, n = 3 for all genotypes ( b , AT100), One-way ANOVA, *** p < 0.001, n = 3 for all genotypes ( b , hTau 421D ) for hTau ( n = 3) vs. hTau plus Vps35 Ri ( n = 3) (Dunnett’s test * p = 0.0361), hTau vs. hTau plus Vps29 Ri ( n = 3) (Dunnett’s test *** p = 0.001), and hTau plus Vps26 Ri ( n = 3) (Dunnett’s test *** p = 0.001). One-way ANOVA, p < 0.001 ( d ) for hTau plus scrambled ( n = 3) vs. hTau plus shRNA-VPS35 ( n = 3) (Dunnett’s test p = 0.4188), hTau plus scrambled vs. hTau plus shRNA-VPS29 ( n = 3) (Dunnett’s test ** p = 0.32), and hTau plus scrambled vs. hTau plus shRNA-VPS26 ( n = 3) (Dunnett’s test *** p < 0.001). Unpaired two-tailed t -test, p = 0.5215, ( f , total hTau) for hTau ( n = 3) vs. hTau plus Dronc Ri ( n = 3), unpaired two-tailed t -test, p < 0.001, ( f , hTau 421D ) for hTau ( n = 3) vs. hTau plus Dronc Ri ( n = 3). Mann–Whitney test, p = 0.4071 for hTau ( n = 16) vs. hTau plus Dronc Ri ( n = 16) ( h , 25 days post induction, n = 18 for control, n = 16 for Dronc Ri ), Mann–Whitney test, *** p < 0.001 for hTau ( n = 20) vs. hTau plus Dronc Ri ( n = 18) ( h , 30 days post induction, n = 20 for control, n = 15 for Dronc Ri ), Mann–Whitney test, *** p < 0.001 for hTau ( n = 20) vs. hTau plus Dronc Ri ( n = 20) ( h , 35 days post induction, n = 17 for control, n = 18 for Dronc Ri ), * p = 0.0396 for hTau ( n = 20) vs. hTau plus Dronc Ri ( n = 20) ( h , 40 days post induction, n = 18 for control, n = 13 for Dronc Ri ), *** p < 0.001 for hTau ( n = 20) vs. hTau plus Dronc Ri ( n = 20) ( h , 45 days post induction, n = 19 for control, n = 15 for Dronc Ri ). n indicates independent biological replicates. Source data are provided as a Source Data file. Full size image To validate the specificity of the effect of retromer depletion upon Tau truncation, we sought to rescue inhibition of Drosophila retromer activity with human transgenes for VPS26A, VPS29, and VPS35. We generated Drosophila transgenes for human retromer components, which due to nucleotide sequence differences, are resistant to inhibition by Drosophila RNAi constructs. We then simultaneously co-expressed these human transgenes together with hTau and the RNAi construct targeting the orthologous Drosophila retromer gene. We found that co-expression of hVPS26A, hVPS29 or hVPS35 significantly reduced the production of truncated hTau 421D when Drosophila retromer components were inhibited (Supplementary Fig. 3a, b ). These results confirmed the specificity of retromer inhibition in Drosophila to enhance the levels of truncated human Tau. We next sought to determine if the effect of retromer depletion on the levels of truncated human Tau was reproducible in an independent human Tau model system. To do this, we utilized a mouse cortical neuron cell line that enables the inducible expression of human Tau [50] (Supplementary Fig. 3c ). Induction of hTau expression in these cells, either alone or together with lentivirus expression of scrambled shRNA constructs results in low levels of hTau 421D production (Fig. 3c and Supplementary Fig. 3c ). However, when murine retromer components were additionally inhibited by lentivirus shRNA expression (Supplementary Fig. 3d ), we observed either a ~7-fold or a 4.5-fold increase in hTau 421D production for mVPS26A or mVPS29, respectively. Levels of hTau 421D were also increased when mVPS35 was inhibited, however, this did not reach statistical significance due to the higher variability of this shRNA construct. In sum, depletion of retromer activity in either Drosophila or murine neuronal cells results in a large increase in the levels of truncated human Tau. Inhibition of the endosomal caspase Dronc reduces Tau truncation and toxicity In mammalian neurons, Tau can be truncated at Aspartate 421 by the activity of Caspases 3, 7, or 8 [46] . To determine the Drosophila Caspase that can cleave human Tau, we employed transgenic RNAi to inhibit the Drosophila caspases Drice, Dredd, and Dronc in animals expressing hTau and measured the levels of hTau 421D produced. We found that inhibition of the caspases Drice and Dredd did not reduce the levels of hTau 421D (Supplementary Fig. 3e, f ). In contrast, inhibition of the caspase Dronc [51] strongly reduced (~6 fold, p < 0.001) the levels of hTau 421D while the total amount of hTau protein was unaffected (Fig. 3e, f ). Dronc, which is present in endosomes [52] , in addition to roles in apoptosis [53] , [54] has also recently been shown to have non-apoptotic functions [55] , [56] , [57] , [58] . Therefore, we tested if inhibition of Dronc could also ameliorate the elevated levels of hTau 421D produced when retromer activity is reduced. Inhibition of Dronc when VPS26 was depleted in the presence of hTau eliminated the increased levels of hTau 421D (Supplementary Fig. 3g, h ) compared to expression of hTau with Vps26 inhibition alone. To further confirm that Dronc could cleave hTau, we also overexpressed a GFP-tagged Dronc construct together with hTau and measured hTau 421D levels. Dronc overexpression induced a significant increase in hTau 421D levels (>2-fold, p < 0.001, Supplementary Fig. 3i, j ) confirming the ability of Dronc to truncate hTau. Therefore, hTau cleavage at Aspartate 421, with or without retromer inhibition, requires the activity of the caspase Dronc. Expanding upon the finding that Dronc is necessary for hTau cleavage at 421D in Drosophila , we next asked if inhibiting this cleavage could alter the toxicity of hTau. When broadly expressed in the adult brain with dTau -Gal4, Dronc RNAi expression alone greatly reduced lifespan (−18.9%, p < 0.001, −7 days survival median Dronc Ri vs control Ri ) compared to control animals (Supplementary Fig. 3k ). Nonetheless, Dronc inhibition in hTau-expressing adults was modestly beneficial resulting in a small, but significant, elongation of lifespan by 4.3% ([ p < 0.001], +1 day median survival hTau & Dronc Ri vs hTau & control Ri ) (Supplementary Fig. 3l ). We then tested the effects of inhibiting Dronc in DC neurons expressing hTau. Axons of DC neurons expressing Dronc Ri alone were unperturbed similar to controls (Fig. 3h ). When Dronc was inhibited together with hTau expression however, this strongly reduced the toxicity of hTau in these neurons, delaying the onset of axonal retraction at Day 30 (32% more axons than hTau alone) such that at this age there was no significant difference to controls (Fig. 3g, h ). The relative preservation of axons persisted throughout lifespan so that at 45 days, three fold more ( p < 0.001) axons were preserved in the medulla when Dronc was simultaneously inhibited compared to hTau expression alone (Fig. 3g, h ). These results demonstrate that the caspase cleavage of Tau is an important contributor to toxicity in these models, suggesting that the accumulation of truncated Tau when retromer is reduced may be essential for exacerbation of Tau toxicity. Increased production of truncated Tau by retromer inhibition is essential for enhanced toxicity To further interrogate if the truncation of Tau is pivotal for the enhanced toxicity when retromer activity is reduced, we generated a transgenic mutant form of hTau where we changed the codon for Aspartate 421 to Glutamate (hTau D421E ), in an approach that has been previously demonstrated to abolish caspase cleavage of hTau at this amino acid [46] . As expected, when we probed for truncated hTau in animals expressing this modified Tau construct, no hTau 421D was detectable (Fig. 4a ). We then used this hTau D421E transgene to test interactions with retromer. When expressed in the eye, similar to wild-type hTau (hTau WT ) hTau D421E also disrupted morphology (Fig. 4b, c ). However, unlike hTau WT expressing animals, when retromer components were simultaneously depleted in animals expressing hTau D421E , we observed no enhancement of toxicity when either VPS35 or VPS29 were inhibited (Fig. 4b, c ). We next evaluated the interaction of retromer depletion with hTau D421E on adult lifespan using dTau-Gal4 expression. Similar to hTau WT , hTau D421E expressing animals have 51.3% ( p < 0.001) shorter median lifespan compared to controls. However, unlike hTau WT , concomitant knock-down of VPS26, VPS29 or VPS35 together with hTau D421E expression did not additionally shorten lifespan (Fig. 4d ). Fig. 4: Abolishing Tau truncation abrogates enhancement of toxicity by retromer inhibition. a Protein analyses of Tau 421D truncated isoform levels in control [GMR-Gal4, UAS-mCD8GFP], hTau expressing [GMR-Gal4, UAS-hTau] and hTau D421E mutant expressing [GMR-Gal4, UAS-hTau D421E ] animals. b Eye morphology of control [GMR-Gal4, UAS-mCD8GFP], hTau D421E expressing [GMR-Gal4, UAS-hTau D421E , UAS-GFP Ri ], and hTau D421E [GMR-Gal4, UAS- hTau D421E ] expression plus inhibition of retromer components [UAS-Vps35 Ri or UAS-Vps29 Ri or UAS-Vps26 Ri ] animals. c Eye disruption scores for control [GMR-Gal4, UAS-mCD8GFP], hTau D421E expressing [GMR-Gal4, UAS-hTau D421E , UAS-GFP Ri ] and hTau D421E [GMR-Gal4, UAS- hTau D421E ] expression plus inhibition of retromer components [UAS-Vps35 Ri or UAS-Vps29 Ri or UAS-Vps26 Ri ] animals. Data are presented as mean values +/− SEM. d Survival analyses of hTau D421E expressing [dTau-Gal4, UAS-hTau D421E , UAS-Cherry Ri , tubulin -Gal80 ts ] and hTau D421E [ dTau -Gal4, UAS-hTau D421E , tubulin -Gal80 ts ] expression together with retromer inhibition [UAS-Vps35 Ri or UAS-Vps29 Ri or UAS-Vps26 Ri ] adults. 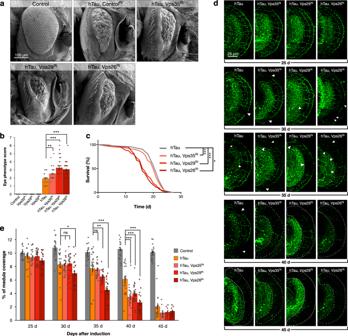Fig. 2: Retromer depletion exacerbates the toxicity of human Tau. aEye morphology in control [GMR-Gal4, UAS-mCD8GFP], hTau expression together with control RNAi [GMR-Gal4, UAS-hTau, UAS-GFPRi] and hTau expression [GMR-Gal4, UAS-hTau] together with RNAi inhibition of retromer components (plus UAS-Vps35Rior UAS-Vps29Rior UAS-Vps26Ri].bEye disruption scores for indicated genotypes. Data are presented as mean values +/− SEM.cSurvival analyses of hTau [dTau-Gal4, UAS-hTau, UAS-CherryRi,tubulin-Gal80ts] and hTau expressing adults [dTau-Gal4, UAS-hTau,tubulin-Gal80ts] together with retromer inhibition [plus UAS-Vps35Rior UAS-Vps29Rior UAS-Vps26Ri].dDC neuron medulla axons with hTau expression alone [ato-Gal4, UAS-hTau, UAS-mCherry, UAS-mCD8GFP,tubulin-Gal80ts] and hTau expression [ato-Gal4, UAS-hTau, UAS-mCherry,tubulin-Gal80ts] together with retromer inhibition [UAS-Vps35Rior UAS-Vps29Rior UAS-Vps26Ri] from 25 to 45 days after onset of transgene expression. Gaps in axonal structure induced by hTau expression are indicated with arrowheads, when <4% axons are present, the medulla is outlined with dashed lines.eQuantification of medulla area occupied by DC neuron axons with hTau expression alone [ato-Gal4, UAS-hTau, UAS-mCherry, UAS-mCD8GFP,tubulin-Gal80ts] and hTau expression [ato-Gal4, UAS-hTau, UAS-mCherry,tubulin-Gal80ts] together with retromer inhibition [UAS-Vps35Rior UAS-Vps29Rior UAS-Vps26Ri] from 25 to 45 days after onset of transgene expression. Data are presented as mean values +/− SEM. Kruskal–Wallis test, ***p< 0.001, for eye disruption scores across all genotypes with multiple comparisons between hTau (n= 34) and hTau plus Vps35Ri(n= 38) (Dunnett’s test **p= 0.003), hTau and hTau plus Vps29Ri(n= 38) (Dunnett’s test ***p< 0.001), and hTau and hTau plus Vps26Ri(n= 29) (Dunnett’s test ***p< 0.001).n= 23 for control,n= 31 for Vps35Ri,n= 30 for Vps29Riandn= 31 for Vps26Ri(b). Mantel-Cox test, ***p= 0.0005 for survival analysis of hTau (n= 148) vs. hTau plus Vps35Ri(n= 153), ***p< 0.001 for hTau vs. hTau plus Vps29Ri(n= 126), and ***p< 0.001 for hTau vs. hTau plus Vps26Ri(n= 173) (c). Kruskal-Wallis test,p= 0.4212 (e, 25 days post induction) for hTau (n= 21) vs. hTau plus Vps35Ri(n= 20) (Dunnett’s testp= 0.9855), hTau vs. hTau plus Vps29Ri(n= 24) (Dunnett’s testp= 0.9999), hTau vs. hTau plus Vps26Ri(n= 18) (Dunnett’s testp= 0.2582),n= 18 for control. Kruskal-Wallis test, *p= 0.0351 (e, 30 days post induction) for hTau (n= 20) vs. hTau plus Vps35Ri(n= 19) (Dunnett’s testp= 0.9974), hTau vs. hTau plus Vps29Ri(n= 20) (Dunnett’s testp= 0.988), hTau vs. hTau plus Vps26Ri(n= 20) (Dunnett’s test *p= 0.0476),n= 20 for control. Kruskal–Wallis test, ***p< 0.001 (e, 35 days post induction) for hTau (n= 20) vs. hTau plus Vps35Ri(n= 20) (Dunnett’s testp= 0.6797), hTau vs. hTau plus Vps29Ri(n= 20) (Dunnett’s test **p= 0.0091), and hTau vs. hTau plus Vps26Ri(n= 22) (Dunnett’s test ***p< 0.001),n= 17 for control. Kruskal-Wallis test, ***p< 0.001 (e, 40 days post induction) for hTau (n= 20) vs. hTau plus Vps35Ri(n= 22) (Dunnett’s test ***p< 0.001), hTau vs. hTau plus Vps29Ri(n= 20) (Dunnett’s test ***p= 0.0005), and hTau vs. hTau plus Vps26Ri(n= 15) (Dunnett’s test ***p< 0.001),n= 18 for control. Kruskal–Wallis test,p= 0.2815 (e, 45 days post induction) for hTau (n= 20) vs. hTau plus Vps35Ri(n= 11) (Dunnett’s testp= 0.1407), hTau vs. hTau plus Vps29Ri(n= 19) (Dunnett’s testp< 0.1209), and hTau vs. hTau plus Vps26Ri(n= 11) (Dunnett’s testp= 0.1728),n= 19 for control. n indicates independent biological replicates. Source data are provided as a Source Data file. e Example DC neuron medulla axons in hTau D421E expressing alone [ ato -Gal4, UAS-hTau D421E , UAS-mCherry, UAS-mCD8GFP, tubulin -Gal80 ts ], and hTau D421E expressing [ ato -Gal4, UAS-hTau D421E , UAS-mCherry, tubulin -Gal80 ts ] together with retromer inhibition [UAS-Vps35 Ri or UAS-Vps29 Ri or UAS-Vps26 Ri ], from 25 to 45 days after onset of transgene expression. Gaps in the axonal structures are indicated with arrowheads. In brains with <4% axons, the medulla is outlined with broken lines. f Quantification of medulla area occupied by DC neuron axons in control [ ato -Gal4, UAS-mCherry, UAS-mCD8GFP, tubulin -Gal80 ts ], hTau D421E expressing alone [ ato -Gal4, UAS-hTau D421E , UAS-mCherry, UAS-mCD8GFP, tubulin -Gal80 ts ], and hTau D421E expressing [ ato -Gal4, UAS-hTau D421E , UAS-mCherry, tubulin -Gal80 ts ] together with retromer inhibition [UAS-Vps35 Ri or UAS-Vps29 Ri or UAS-Vps26 Ri ]. Data are presented as mean values +/− SEM. Kruskal–Wallis test, p = 0.3272 for eye disruption scores across all genotypes with multiple comparisons between hTau D421E ( n = 33) and hTau D421E plus Vps35 Ri ( n = 30) (Dunnett’s test p = 0.1716), hTau D421E and hTau D421E plus Vps29 Ri ( n = 31) (Dunnett’s test p = 0.5443), and hTau D421E and hTau D421E plus Vps26 Ri ( n = 29) (Dunnett’s test p = 0.9899), n = 32 for control ( c ). Mantel-Cox test, p = 0.2508 for survival analysis of hTau D421E ( n = 248) vs. hTau D421E plus Vps35 Ri ( n = 218), * p = 0.0105 for hTau D421E vs. hTau D421E plus Vps29 Ri ( n = 233), and p = 0.0988 for hTau D421E and hTau D421E plus Vps26 Ri ( n = 260) ( d ). Kruskal–Wallis test, p = 0.9847 ( f , 25 days post induction) with multiple comparisons between hTau D421E ( n = 20) and hTau D421E plus Vps35 Ri ( n = 19) (Dunnett’s test p = 0.9873), hTau D421E and hTau D421E plus Vps29 Ri ( n = 20) (Dunnett’s test p = 0.9557), and hTau D421E and hTau D421E plus Vps26 Ri ( n = 18) (Dunnett’s test p = 0.9999), n = 18 for control. Kruskal–Wallis test, p = 0.9552 ( f , 30 days post induction), with multiple comparisons between hTau D421E ( n = 19) and hTau D421E plus Vps35 Ri ( n = 16) (Dunnett’s test p = 0.9991), hTau D421E and hTau D421E plus Vps29 Ri ( n = 20) (Dunnett’s test p = 0.9999), and hTau D421E plus Vps26 Ri ( n = 18) (Dunnett’s test p = 0.9714), n = 20 for control. Kruskal-Wallis test, p = 0.4127 ( f , 35 days post induction), with multiple comparisons between hTau D421E ( n = 18) and hTau D421E plus Vps35 Ri ( n = 16) (Dunnett’s test p = 0.5464), hTau D421E and hTau D421E plus Vps29 Ri ( n = 20) (Dunnett’s test p = 0.8007), and hTau D421E plus Vps26 Ri ( n = 19) (Dunnett’s test p = 0.4417), n = 17 for control. Kruskal–Wallis test, * p = 0.0127 ( f , 40 days post induction), with multiple comparisons between hTau D421E ( n = 19) and hTau D421E plus Vps35 Ri ( n = 20) (Dunnett’s test p = 0.108), hTau D421E and hTau D421E plus Vps29 Ri ( n = 19) (Dunnett’s test p = 0.111), and hTau D421E plus Vps26 Ri ( n = 19) (Dunnett’s test ** p = 0.0013), n = 18 for control. Kruskal–Wallis test, p = 0.4553 ( f , 45 days post induction), with multiple comparisons between hTau D421E ( n = 20) and hTau D421E plus Vps35 Ri ( n = 11) (Dunnett’s test p = 0.2311), hTau D421E and hTau D421E plus Vps29 Ri ( n = 13) (Dunnett’s test p = 0.3127), and hTau D421E plus Vps26 Ri ( n = 20) (Dunnett’s test ** p = 0.1683), n = 19 for control. n indicates independent biological replicates. Source data are provided as a Source Data file. Full size image We next expressed hTau D421E in adult DC neurons. Again, similar to expression of hTau WT , expression of hTau D421E in adult DC neurons induced progressive loss of axons over time (Fig. 4e, f ). However, simultaneous inhibition of VPS26 and VPS29 did not accelerate or increase this loss at any time point. This was also the case for all timepoints when VPS26 was inhibited together with hTau D421E expression, apart from measurements at 40 days after induction, where we did observe a small but significant additional loss of axons when VPS26 was inhibited (Fig. 4e, f ), though the magnitude of this loss was less (18% less, p < 0.01) than that observed with hTau WT expression (Fig. 2d, e ). Therefore, not only does depletion of retromer activity induce a large accumulation of truncated human Tau, but inhibition of the production of this truncated isoform, either by mutating the Tau cleavage site or by inhibiting the essential caspase, abrogates the increased toxicity of Tau when retromer is reduced. Conceivably, the increased accumulation of hTau 421D that we observe when retromer function is inhibited could be the result of an increase in the production of truncated Tau molecules or from a failure to appropriately process and degrade existing truncated Tau species. To differentiate between these models, we next generated Drosophila lines that express hTau with a stop codon after Aspartate 421 [hTau 421X ] so the entirety of hTau in these animals was truncated. Consistent with prior observations, we found this truncated isoform of hTau was highly toxic [8] , [47] , so for interaction studies we generated transgenic lines that produce lower levels of hTau 421X than the equivalent full length hTau lines. Nonetheless, this lower amount of transgenic hTau 421X expression resulted in a strong disruption of eye morphology equivalent to expression of higher levels of full length hTau (Fig. 5a ). In these animals, we then inhibited retromer activity. We found that in contrast to animals expressing full length hTau, we observed no increased disruption of eye morphology when we inhibited VPS35, VPS29 or VPS35 in the context of hTau 421X expression (Fig. 5a, b ). Furthermore, when we examined the levels of truncated Tau protein present in these animals, we found no increase when retromer was inhibited compared to transgenic hTau 421X expression alone (Fig. 5c ). These data are consistent with the reduction of retromer activity increasing the production of truncated Tau from full length Tau rather than a reduced ability to remove this truncated species. Fig. 5: The toxicity of extant truncated Tau is not enhanced by retromer depletion. a Eyes from control [GMR-Gal4, UAS-mCD8GFP], hTau 421X expressing [GMR-Gal4, UAS-hTau 421X , UAS-GFP Ri ] animals, and hTau 421X [GMR-Gal4, UAS-hTau 421X ] expressing together with retromer inhibition [UAS-Vps35 Ri or UAS-Vps29 Ri or UAS-Vps26 Ri ] animals. b Eye disruption scores for control [GMR-Gal4, UAS-mCD8GFP], hTau 421X expressing [GMR-Gal4, UAS-hTau 421X , UAS-GFP Ri ] animals, and hTau 421X [GMR-Gal4, UAS-hTau 421X ] expressing together with retromer inhibition [UAS-Vps35 Ri or UAS-Vps29 Ri or UAS-Vps26 Ri ] animals. Data are presented as mean values +/− SEM. c Truncated Tau (hTau 421D ) levels from head lysates of control [GMR-Gal4, UAS-mCD8GFP], hTau 421X expressing [GMR-Gal4, UAS-hTau 421X , UAS-GFP Ri ], and hTau 421X expressing [GMR-Gal4, UAS-hTau 421X ] together with retromer inhibition [UAS-Vps35 Ri or UAS-Vps29 Ri or UAS-Vps26 Ri ] animals. Kruskal–Wallis test, p = 0.8297 for eye disruption scores across all genotypes with multiple comparisons between hTau 421X ( n = 30) and hTau 421X plus Vps35 Ri ( n = 30) (Dunnett’s test p = 0.8779), hTau 421X and hTau 421X plus Vps29 Ri ( n = 32) (Dunnett’s test p = 0.9999), and hTau 421X and hTau 421X plus Vps26 Ri ( n = 31) (Dunnett’s test p = 0.564). n indicates independent biological replicates. Source data are provided as a Source Data file. Full size image Diminished interaction of Retromer with Rab7 leads to an accumulation of truncated Tau in late endosomes As the increased production of hTau 421D was critical to the enhancement of hTau toxicity by retromer depletion, we next sought to investigate the localization of this species of Tau within neurons with single cell resolution. To do this, we labeled a small subset of glutamatergic neurons in the Drosophila nervous system characterized by the expression of the transcription factor dHB9 [59] , [60] having confirmed these neurons also express dTau (Supplementary Fig. 4a ). Next, we expressed hTau in dHb9 neurons and examined the intracellular localization of full-length and truncated hTau. While full-length hTau was distributed throughout the neuron (Supplementary Fig. 4b ), hTau 421D was localized to discrete compartments within both the neuron axon and soma (Fig. 6a, b ). We assessed the nature of these compartments using markers specific for intracellular trafficking organelles. We observed poor localization with markers for many organelles including early endosomes labeled by Rab4 and Rab5 (Supplementary Fig. 4c, d ). However, we did observe encapsulation of hTau 421D accumulations within compartments labeled by Rab7, a marker of late endosomes (Fig. 6c , Supplementary Movie 1 ). We quantified this spatial relationship using Manders analysis [61] (Fig. 6d ). We examined the overlap of hTau 421D with Rab4, Rab5 and Rab7 labeled compartments. We found no significant overlap of hTau 421D between Rab4 and Rab5 compartments. In contrast, the overlap between hTau 421D and Rab7 compartments was highly significant ( p < 0.001). This indicated hTau 421D accumulations were largely within Rab7 labeled late endosomes. We also examined if hTau 421D accumulated in DC neurons (Supplementary Fig. 4e ). Similar to HB9 neurons, when hTau was expressed in DC neurons, we also observed hTau 421D accumulations in Rab7 labeled compartments within their soma (Supplementary Fig. 4f ). Interestingly, a recent report has also demonstrated colocalization of hTau 421D with Rab7 in postmortem brains of AD patients [62] . Fig. 6: Reduction of Retromer leads to accumulation of truncated Tau in late endosomes. a , b Left panel: Soma and axons of dHB9 neurons expressing hTau and mCherry (blue) [ dHB9 -Gal4, UAS-hTau, UAS-mCherry, UAS-mCD8GFP]. hTau 421D (green) accumulates in discrete subcellular compartments. Right panels: hTau 421D accumulations labeled by arrowheads. c Left panel: hTau 421D (green) encapsulated in late endosomal compartments labeled with Rab7-GFP (red) in the soma of dHB9 expressing hTau neurons [ dHB9 -Gal4, UAS-hTau, UAS-Rab7-GFP, UAS-mCherry]. Middle panel: hTau 421D accumulations labeled by arrowheads. Right panel: Rab7-GFP (red), hTau 421D (green) and mCherry (blue). d Mander’s analyses of the spatial relationship of hTau 421D with endosomes labeled by either Rab4-GFP ( n = 12), Rab5-GFP ( n = 12) or Rab7-GFP ( n = 11). M1 is the fraction of each Rab protein overlapping with Tau 421D , while M2 is the fraction of Tau 421D signal overlapping with each Rab protein signal. e , f Left panels: hTau 421D accumulations (green) in the soma ( e ) and axons ( f ) of hHB9 neurons (mCherry, blue) expressing hTau together with retromer inhibition [ dHB9 -Gal4, UAS-hTau, UAS-Vps26 Ri , UAS-mCherry]. Right panels: hTau 421D accumulations labeled by arrowheads. g Relative area of hTau 421D accumulations normalized to neuronal area in dHB9 neurons expressing hTau [ dHB9 -Gal4, UAS-hTau, UAS-mCherry, UAS-mCD8GFP] and when retromer is inhibited [ dHB9 -Gal4, UAS-hTau, UAS-mCherry, UAS-Vps26 Ri ]. Data are presented as mean values +/− SEM. h Intensity of hTau 421D accumulations normalized to mCherry in dHB9 neurons expressing hTau [ dHB9 -Gal4, UAS-hTau, UAS-mCherry, UAS-mCD8GFP] and when retromer is inhibited [ dHB9 -Gal4, UAS-hTau, UAS-mCherry, UAS-Vps26 Ri ]. Data are presented as mean values +/− SEM. i Left panel: hTau 421D (green) encapsulated in late endosomal compartments labeled with Rab7-GFP (red) in the soma of dHB9 expressing hTau neurons when retromer is inhibited [ dHB9 -Gal4, UAS-hTau, UAS-Rab7-GFP, UAS-mCherry, UAS-Vps26 Ri ]. Middle panel: hTau 421D accumulations labeled by arrowheads. Right panel: Rab7-GFP (red), hTau 421D (green) and mCherry (blue). Unpaired two-tailed t -test, ***p < 0.001, hTau vs. hTau plus Vps26 Ri ( n = 11 neurons examined over three independent experiments) ( g ). Unpaired two-tailed t -test, **p = 0.0039, hTau vs. hTau plus Vps26 Ri ( n = 11 neurons examined over three independent experiments) ( h ). n indicates independent biological replicates. Source data are provided as a Source Data file. Full size image We next examined the levels and localization of hTau 421D in neurons when retromer was depleted. We observed a dramatic increase in the immunohistochemical levels of hTau 421D (Fig. 6e, f ), consistent with our protein blot measurements (Fig. 3e, f ). We quantified this increase and found hTau 421D levels increased in area by 3.5-fold ( p < 0.001) per neuron and in intensity by 2.5-fold ( p < 0.01) per neuron when VPS26 was inhibited compared to neurons which express hTau alone (Fig. 6g, h ). Like neurons expressing hTau alone, the increased accumulations of hTau 421D when retromer was inhibited were also restricted to Rab7 labeled late endosomes (Fig. 6i ). Rab7 has previously been shown to interact directly with the retromer complex [40] , suggesting the possibility that hTau 421D might be accumulating in late endosomes due to a diminishment of this interaction. To test this hypothesis, we first confirmed using co-immunoprecipitation that Drosophila Rab7 could indeed interact with Drosophila VPS35 in vivo (Supplementary Fig. 5a ). We also confirmed that this interaction did not occur with a ‘GDP-locked’ mutant version of Rab7 [Rab7 T22N ] (Supplementary Fig. 5a ), sometimes known as ‘Dominant-Negative’ Rab7 [63] , [64] . Having validated that retromer and Rab7 biochemically interact in Drosophila , we next wished to investigate if modulation of Rab7 activity could also alter hTau truncation. To deplete Rab7, we used deGradFP nanobodies [65] to degrade Rab7 tagged in-frame with YFP inserted into the endogenous genetic locus [66] . We confirmed expression of deGradFP nanobodies throughout the brain could deplete Rab7 levels by 87% ( p < 0.001) (Supplementary Fig. 5b, c ). We next combined this method of Rab7 depletion with simultaneous expression of hTau. We found that depletion of Rab7 resulted in a ~6-fold ( p < 0.001) increase in the levels of hTau 421D compared to hTau expression alone (Fig. 7a, b ). To confirm this result, we also examined animals where GDP-locked Rab7 T22N was co-expressed with hTau. Similar to depletion of Rab7, expression of Rab7 T22N with hTau resulted in a ~5-fold ( p < 0.001) increase of hTau 421D levels (Fig. 7a, b ). In contrast, co-expression of either wildtype Rab7 or a ‘GTP-locked’ mutant Rab7 [Rab7 Q67L ] [63] with hTau did not significantly alter truncated Tau levels (Supplementary Fig. 5d, e ). We additionally confirmed that, similar to retromer inhibition, accumulation of hTau 421D when Rab7 was inhibited also required Dronc caspase activity (Supplementary Fig. 5f, g ) and that levels of hTau 421D were not changed when hTau 421X was expressed together with Rab7 inhibition (Supplementary Fig. 5h ). Therefore, inhibition of Rab7, like inhibition of retromer, results in increased production (and not clearance) of truncated Tau. Fig. 7: Rab7 inhibition increases Tau truncation. a hTau 421D protein level analyses from head lysates of controls [GMR-Gal4, UAS-mCD8GFP], hTau expressing [GMR-Gal4, UAS-hTau, UAS-DeGradFP] and hTau expressing together with Rab7 knock-down (Rab7 KD ) [GMR-Gal4, UAS-hTau, Rab7 EYFP/ΔRab7 , UAS-DeGradFP] or Rab7 T22N expression [GMR-Gal4, UAS-hTau, UAS-Rab7 T22N ] animals. b Quantification of hTau 421D protein levels from head lysates of controls [GMR-Gal4, UAS-mCD8GFP], hTau expressing [GMR-Gal4, UAS-hTau, UAS-DeGradFP] and hTau expressing together with Rab7 knock-down (Rab7 KD ) [GMR-Gal4, UAS-hTau, Rab7 EYFP/ΔRab7 , UAS-DeGradFP] or Rab7 T22N expression [GMR-Gal4, UAS-hTau, UAS-Rab7 T22N ] animals. Data are presented as mean values +/− SEM. c Eyes from control [GMR-Gal4, UAS-mCD8GFP], hTau expressing [GMR-Gal4, UAS-hTau, UAS-mCD8GFP], Rab7 knockdown alone (Rab7 KD ) [GMR-Gal4, Rab7 EYFP/ΔRab7 , UAS-DeGradFP], hTau expressing with Rab7 KD [GMR-Gal4, UAS-hTau, Rab7 EYFP/ΔRab7 , UAS-DeGradFP], Rab7 inhibition (Rab7 T22N ) alone [GMR-Gal4, UAS-Rab7 T22N , UAS-mCD8GFP], and hTau expression together with Rab7 T22N [GMR-Gal4, UAS-hTau, UAS-Rab7 T22N ] animals. d Eye disruption scores from control [GMR-Gal4, UAS-mCD8GFP], hTau expressing [GMR-Gal4, UAS-hTau, UAS-DeGradFP], Rab7 KD [GMR-Gal4, Rab7 EYFP/ΔRab7 , UAS-DeGradFP], hTau expressing with Rab7 KD [GMR-Gal4, UAS-hTau, Rab7 EYFP/ΔRab7 , UAS-DeGradFP], Rab7 T22N [GMR-Gal4, UAS-Rab7 T22N , UAS-mCD8GFP], and hTau expression together with Rab7 T22N [GMR-Gal4, UAS-hTau, UAS-Rab7 T22N ] animals. Data are presented as mean values +/− SEM. e Example DC neuron medulla axons from control [ ato -Gal4, UAS-mCherry, UAS-mCD8GFP, tubulin -Gal80 ts ], Rab7 T22N expression alone [ ato -Gal4, UAS-Rab7 T22N , UAS-mCherry, tubulin -Gal80 ts ], hTau expression alone [ ato -Gal4, UAS-hTau, UAS-mCherry, UAS-mCD8GFP, tubulin -Gal80 ts ], and hTau expression together with Rab7 inhibition [ ato -Gal4, UAS-hTau, UAS-Rab7 T22N , UAS-mCherry, tubulin -Gal80 ts ] animals from 20 to 45 days after onset of transgene expression. Gaps in axonal structure induced by hTau expression are indicated with arrowheads, when < 4% axons are present, the medulla is outlined with dashed lines. f Quantification of medulla area occupied by DC neuron from control [ ato -Gal4, UAS-mCherry, UAS-mCD8GFP, tubulin -Gal80 ts ], Rab7 T22N expression alone [ ato -Gal4, UAS-Rab7 T22N , UAS-mCherry, tubulin -Gal80 ts ], hTau expression alone [ ato -Gal4, UAS-hTau, UAS-mCherry, UAS-mCD8GFP, tubulin -Gal80 ts ], and hTau expression together with Rab7 inhibition [ ato -Gal4, UAS-hTau, UAS-Rab7 T22N , UAS-mCherry, tubulin -Gal80 ts ] 20–45 days after onset of transgene expression. Data are presented as mean values +/− SEM. Unpaired two-tailed t -test, p < 0.001, ( b , hTau 421D ) for hTau ( n = 3) vs. hTau plus Rab7 KD ( n = 3), and p < 0.001 for hTau ( n = 3) vs. hTau plus Rab7 T22N ( n = 3). Kruskal–Wallis test, *** p < 0.001 for eye disruption scores across all genotypes with multiple comparisons between hTau ( n = 26) and hTau plus Rab7 KD ( n = 26) (Dunnett’s test *** p < 0.001), and hTau and hTau plus Rab7 T22N ( n = 28). n = 32 for control, n = 30 for Rab7 KD , and n = 28 for Rab7 T22N ( d ). Mann–Whitney test, p = 0.2928 for hTau ( n = 15) vs. hTau plus Rab7 T22N ( n = 18) ( f , 20 days post induction, n = 15 for control and n = 16 for Rab7 T22N ). Mann–Whitney test, *** p < 0.001 for hTau ( n = 16) vs. hTau plus Rab7 T22N ( n = 15) ( f , 25 days post induction, n = 18 for control and n = 17 for Rab7 T22N ). Mann–Whitney test, *** p < 0.001 for hTau ( n = 20) vs. hTau plus Rab7 T22N ( n = 17) ( f , 30 days post induction, n = 20 for control and n = 15 for Rab7 T22N ). Mann–Whitney test, *** p < 0.001 for hTau ( n = 20) vs. hTau plus Rab7 T22N ( n = 18) ( f , 35 days post induction, n = 17 for control and n = 15 for Rab7 T22N ). Mann–Whitney test, *** p < 0.001 for hTau ( n = 20) vs. hTau plus Rab7 T22N ( n = 12) ( f , 40 days post induction, n = 18 for control and n = 14 for Rab7 T22N ). Mann–Whitney test, p = 0.7132 for hTau ( n = 20) vs. hTau plus Rab7 T22N ( n = 10) ( f , 45 days post induction, n = 19 for control and n = 14 for Rab7 T22N ). n indicates independent biological replicates. Source data are provided as a Source Data file. Full size image We then examined if phenotypes produced by hTau expression were altered when Rab7 activity was inhibited. Depletion of Rab7 using the nanobody approach had no effect on eye morphology (Fig. 7c, d ). However, depletion of Rab7 together with hTau expression resulted in a 41.3% ( p < 0.001) increase of the disruption of eye morphology compared to hTau expression alone. Expression of Rab7 T22N did modestly alter eye morphology when expressed alone (Fig. 7c, d ), but co-expression with hTau also increased morphological disruption by 45.2% ( p < 0.001) compared to hTau expression alone (Fig. 7c, d ). In contrast, co-expression of Rab7 T22N together with cleavage-resistant hTau D421E or truncated hTau 421X did not result in any additional disruption to eye morphology (Supplementary Fig. 6a, b, c ). Expression of Rab7 WT or Rab7 Q67L also failed to additionally alter eye morphology when co-expressed with hTau (Supplementary Fig. 6d, e ). Thus, inhibition of Rab7, similar to retromer, increases the hTau-dependent disruption of eye morphology consistent with a specific increase in the production of truncated Tau. We then examined the effects of Rab7 inhibition in lifespan. Expression of Rab7 T22N with dTau-Gal4 modestly reduced lifespan (−8%, p < 0.001) (Supplementary Fig. 6f ). However, expression of Rab7 T22N with hTau additionally reduced lifespan by −13.6% ( p < 0.001) compared to hTau expression alone (Supplementary Fig. 6g ). Finally, we examined the effects of Rab7 inhibition on DC neuron degeneration. Expression of Rab7 T22N alone in DC neurons did not significantly affect medulla axons during early life though we did observe a modest but significant decline of axons after 35 days (Fig. 7e, f ). In contrast, inhibition of Rab7 together with hTau resulted in a large increase in axonal loss compared to expression of hTau alone beginning from 25 days onwards (+48.3% at 25d, +60.8% at 30d, +82% at 35d, +79% at 40d [ p < 0.001]). This acceleration was such that, after 35 days, almost all axons were lost in contrast to hTau expression alone (Fig. 7e, f ). Therefore, in these assays, consistent with our observation of increased truncated Tau production, inhibition of Rab7, just as with depletion of retromer, increases the toxicity of human Tau expression. Our results support that the association of retromer with Rab7 is essential for the late endosomal trafficking of Tau and that disruption of either partner results in the accumulation of toxic truncated Tau species. Deposition of abnormal, aggregated species of Tau protein is a characteristic feature of many neurodegenerative diseases [6] . In particular, Tau truncated at the C-terminus is both highly fibrillogenic and prone to aggregation [8] , [67] , [68] , [69] , [70] . One of these neurotoxic forms of Tau, Tau 421D , is cleaved at Aspartate 421 by caspase activity [46] , [71] , [72] , [73] , [74] . Tau 421D truncation enhances the polymerization rate of Tau [43] , [68] , [70] and this isoform is abundant in neurofibrillary tangles in both AD brains and those of other tauopathies [46] , [75] , [76] . Here, we show using models for human Tau toxicity in Drosophila , and recapitulated in mammalian neurons, that reduction of retromer activity amplifies the toxicity of human Tau expression upon both neuronal degeneration and animal viability in tandem with a specific and dramatic increase in the abundance of Tau 421D . We show that this truncated form of Tau accumulates in neuronal late endosomes and establish that activity of the late endosome protein and retromer partner Rab7 is also essential to prevent accumulation of this truncated Tau species. Our data suggest a mechanism (Fig. 8 ) whereby depletion of retromer levels in neurons results in reduced retromer/Rab7 complexes. The endosomal trafficking of Tau, which can enter the network via endocytosis [77] or autophagy [10] , [43] , [78] , [79] en route to the lysosome [63] , is abnormally protracted by this depletion of retromer/Rab7 activity. This retardation of the endosomal flow of Tau extends exposure to caspases, such as human Caspases 3, 7 or 8 [46] or Drosophila Dronc [51] , [52] , active within the endosomal/lysosomal network [7] resulting in abnormally enhanced levels of truncation. The resulting aberrant abundance of neurotoxic truncated Tau is detrimental to synapse and axon stability and ultimately animal viability. Fig. 8: Model for enhancement of Tau toxicity and truncation by retromer depletion. In wildtype neurons full length Tau (orange) enters the endosomal network and is efficiently trafficked through the late endosome to the lysosome enabled by the interaction of the retromer complex (yellow) with the late endosome protein Rab7 (blue). When retromer or Rab7 activity is reduced, endosomal-lysosomal flux is retarded, exposing Tau to endosomal resident caspase activity which results in Tau truncation (red) and accumulation in the late endosome. Truncation of Tau enhances its neurotoxicity. Full size image Our evidence supports that the increased production of Tau 421D is singularly critical for and causal of the enhancement of Tau toxicity upon retromer deficiency. Firstly, while Tau truncation is dramatically increased when retromer levels are depleted, the levels of total Tau or several phosphorylated forms of Tau were unchanged, although potentially some additional Tau phosphoepitopes we did not examine could show alterations or perhaps some alterations were below our detection limit. Second, even though other modifications of Tau could occur [80] , inhibition of the caspase Dronc, which we show is necessary for cleavage of human Tau at Aspartate 421 in Drosophila , eliminates the enhancement of Tau toxicity by retromer depletion. Third, mutation of Aspartate 421 (hTau D421E ) in human Tau also abrogates the amplification of Tau toxicity by retromer depletion. Finally, the toxicity of Tau already truncated at Aspartate 421 is not further increased by depletion of retromer activity. This latter result additionally establishes that retromer depletion increases the production of Tau 421D rather than perturbing the ability of neurons to eliminate this species. Similar results and specificity of Tau 421D production were established when Rab7 was depleted. Even in the absence of truncation, for example with hTau D421E expression, elevated human Tau expression remains toxic to Drosophila , indicating this cleavage event is not solely responsible for all the detrimental effects of Tau in this model. But the results above in our models, together with the observed heightened toxicity of truncated Tau (e.g., hTau 421X expression), establish that Tau truncation is both necessary and sufficient to explain the intensification of Tau neurotoxicity in response to retromer depletion. Interaction of the retromer complex with endosomal compartments, through either Rab5 or Rab7 proteins, is essential for the normal function of the endosomal-lysosomal pathway [81] , [82] . Trafficking in endosomal-lysosomal network is responsible for many key cellular processes including protein recycling and degradation, cellular signaling, and nutrient uptake [82] . Disruption of the endosomal-lysosomal system has been implicated in the pathology of several neurodegenerative diseases including AD [81] . The initial processing of Amyloid-beta precursor protein (APP), the precursor of Amyloid-beta plaques [83] , takes place within endosomes and pathological increases of amyloid-beta are dependent upon prolonged APP residence within endosomal compartments [81] . Consistent with a role for endosomal dysfunction in AD, endosomal compartments are enlarged in postmortem AD brains [84] , [85] , congruous with a retardation of endosomal-lysosomal flux [85] . Disease-specific lysosomal truncation of α-synuclein has been shown to occur in the brains of PD patients [86] and Tau, like APP and α-synuclein, is also subject to processing and degradation via the endosomal-lysosomal system [79] . Mutations in the retromer component VPS35 are linked to familial Parkinson’s disease [17] , [18] , [19] , [20] , [21] , [22] and cause an enlargement of endosomes [82] , consistent with a ‘traffic jam’ within the endosomal-lysosomal system [85] . In addition, the familial PD linked protein LRRK2 [87] , [88] has also been implicated in the aberrant processing of α-Synuclein through interaction with the Rab7 related protein PARK16/Rab7L1. Reduced retromer interaction with the endosomal network can also cause increased processing of APP into amyloid-beta [18] , though it is noteworthy that Drosophila do not produce Aβ in the absence of transgenic human BACE [89] , allowing us to exclude the effects we observe upon Tau toxicity with retromer depletion in our assays as a potentially indirect consequence of the modification of Aβ [29] in our models. Consistent with our findings, recent studies have also shown that retromer-deficient cells have inhibited autophagic flux which can promote Tau aggregation [79] and that Tau neuropathology is evident in mice harboring Parkinson’s disease-associated VPS35 mutations [90] . Our data support that hampered endosomal-lysosomal flux of Tau in retromer or Rab7 deficient neurons promotes the aberrant production of neurotoxic truncated species through prolonged exposure to endosomal resident caspases. Therefore, deficits in endosomal-lysosomal flux, a common feature in several neurodegenerative diseases, could contribute to protein processing dysfunction at multiple junctures. The exploitation of Drosophila genetic models to study human neurodegenerative diseases has provided several insights into disease mechanisms [91] . Expression of disease-related proteins in the developing eye provides an easy-to-score and high-throughput assay to establish the relative toxicity of disease-associated moieties and to identify genetic or chemical modifiers [33] , [91] , [92] . Here we introduce a Drosophila model system that enables adult restricted expression of disease-associated proteins within a sparse and highly reproducible subset of CNS neurons. This assay enables the visualization and quantification of some of the earliest features of neurodegeneration, namely synapse loss and axonal retraction, with single neuron resolution within the context of an intact functioning brain and animal. This system enabled us to identify the differential effects of retromer depletion upon the earliest consequences to synapses and axons of Tau expression. Moreover, it enabled assays, such as assessment of the effect of inhibition of the caspase Dronc upon Tau truncation, and the consequent benefits to axon preservation, that would have been potentially obscured by the pleiotropic effects of broader manipulations. 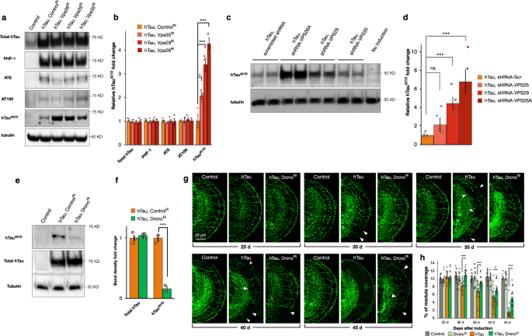Fig. 3: Human Tau truncation requires the caspase Dronc. ahTau protein analyses from head lysates of controls [GMR-Gal4, UAS-mCD8GFP], hTau expressing animals [GMR-Gal4, UAS-hTau, UAS-GFPRi], and hTau [GMR-Gal4, UAS-hTau] expression together with retromer inhibition [UAS-Vps35Rior UAS-Vps29Rior UAS-Vps26Ri].bQuantification of total Tau protein levels, Tau phosphorylation (PHF-1, AT8, and AT100) or truncation (Tau421D). Data are presented as mean values +/− SEM.cProtein analyses of truncated Tau levels in CN1.4 mouse cortical neurons expressing inducible full-length human Tau (0N4R) and scrambled shRNA or shRNAs against murine VPS26A, or VPS29, or VPS35.dQuantification of truncated Tau levels in CN1.4 neurons expressing human Tau and scrambled shRNA or shRNAs against murine VPS26A, or VPS29, or VPS35. Data are presented as mean values +/− SEM.eProtein analyses of head lysates from control [GMR-Gal4, UAS-mCD8GFP], hTau expressing [GMR-Gal4, UAS-hTau, UAS-GFPRi] animals, and hTau expression together with Dronc inhibition [GMR-Gal4, UAS-hTau, UAS-DroncRi], probed with anti-hTau421D(top) or anti-total Tau [TauC] (middle).fQuantification of total and truncated Tau levels from RNAi control [GMR-Gal4, UAS-hTau, UAS-GFPRi] animals and hTau expression together with Dronc inhibition [GMR-Gal4, UAS-hTau, UAS-DroncRi]. Data are presented as mean values +/− SEM.gDC neuron medulla axons in control [ato-Gal4, UAS-mCherry, UAS-mCD8GFP,tubulin-Gal80ts], hTau expressing [ato-Gal4, UAS-hTau, UAS-mCherry, UAS-mCD8GFP,tubulin-Gal80ts] animals, and hTau expression together with Dronc inhibition [ato-Gal4, UAS-hTau, UAS-DroncRi, UAS-mCherry,tubulin-Gal80ts] from 25 to 45 days after onset of transgene expression.hQuantification of medulla area occupied by DC neuron control [ato-Gal4, UAS-mCherry, UAS-mCD8GFP,tubulin-Gal80ts], hTau expressing [ato-Gal4, UAS-hTau, UAS-mCherry, UAS-mCD8GFP,tubulin-Gal80ts] animals, and hTau expression together with Dronc inhibition [ato-Gal4, UAS-hTau, UAS-DroncRi, UAS-mCherry,tubulin-Gal80ts] from 25 to 45 days after onset of transgene expression. Data are presented as mean values +/− SEM. One-Way ANOVA,p= 0.5466,n= 3 for all genotypes (b, total hTau), One-way ANOVA,p= 0.8216,n= 3 for all genotypes (b, PHF-1), One-way ANOVA,p= 0.8216n= 3 for all genotypes, (b, PHF-1), One-way ANOVA,p= 0.8791,n= 3 for all genotypes (b, AT8), One-Way ANOVA,p= 0.8982,n= 3 for all genotypes (b, AT100), One-way ANOVA, ***p< 0.001,n= 3 for all genotypes (b, hTau421D) for hTau (n= 3) vs. hTau plus Vps35Ri(n= 3) (Dunnett’s test *p= 0.0361), hTau vs. hTau plus Vps29Ri(n= 3) (Dunnett’s test ***p= 0.001), and hTau plus Vps26Ri(n= 3) (Dunnett’s test ***p= 0.001). One-way ANOVA,p< 0.001 (d) for hTau plus scrambled (n= 3) vs. hTau plus shRNA-VPS35 (n= 3) (Dunnett’s testp= 0.4188), hTau plus scrambled vs. hTau plus shRNA-VPS29 (n= 3) (Dunnett’s test **p= 0.32), and hTau plus scrambled vs. hTau plus shRNA-VPS26 (n= 3) (Dunnett’s test ***p< 0.001). Unpaired two-tailedt-test,p= 0.5215, (f, total hTau) for hTau (n= 3) vs. hTau plus DroncRi(n= 3), unpaired two-tailedt-test,p< 0.001, (f, hTau421D) for hTau (n= 3) vs. hTau plus DroncRi(n= 3). Mann–Whitney test,p= 0.4071 for hTau (n= 16) vs. hTau plus DroncRi(n= 16) (h, 25 days post induction,n= 18 for control,n= 16 for DroncRi), Mann–Whitney test, ***p< 0.001 for hTau (n= 20) vs. hTau plus DroncRi(n= 18) (h, 30 days post induction,n= 20 for control,n= 15 for DroncRi), Mann–Whitney test, ***p< 0.001 for hTau (n= 20) vs. hTau plus DroncRi(n= 20) (h, 35 days post induction,n= 17 for control,n= 18 for DroncRi), *p= 0.0396 for hTau (n= 20) vs. hTau plus DroncRi(n= 20) (h, 40 days post induction,n= 18 for control,n= 13 for DroncRi), ***p< 0.001 for hTau (n= 20) vs. hTau plus DroncRi(n= 20) (h, 45 days post induction,n= 19 for control,n= 15 for DroncRi).nindicates independent biological replicates. Source data are provided as a Source Data file. We envision this new model system, coupled with the automated tools we have developed to enable precise quantification of CNS synapse and axonal degeneration, will enable additional mechanistic insights into the intricate web of interactions between factors associated with susceptibility to human neurodegenerative disease. Drosophila strains UAS-hTau [2N4R] was described previously [32] . To generate UAS-hTau-421X, a stop codon was inserted to replace Serine 422 in hTau using KLD Enzyme Mix (New England Biolabs) and transgenes generated using pBID [93] Drosophila expression vector. To inhibit retromer components we used UAS-RNAi-Vps35 [94] (BDSC# 38944), UAS-RNAi-Vps29 [94] (BDSC# 38963) and UAS-RNAi-Vps26 [94] (BDSC# 38937). For protein interactions with retromer we used UAS-Vps35HA [95] and UAS-Vps29-HA [96] . To manipulate Rab7 we used UAS-Rab7-GFP (BDSC# 42705 and 42706), UAS-YFP-Rab7 [T22N] [97] (BDSC# 23235), UAS-Venus-Rab7 [WT] [98] and UAS-Venus-Rab7 [T22N] [98] . For eye expression we employed GMR-Gal4 [99] , for DC neuron expression ato -Gal4[14a] [38] , and for whole brain expression Elav-Gal4 [100] (BDSC# 458). Additional strains and procedures are described in supplemental methods. 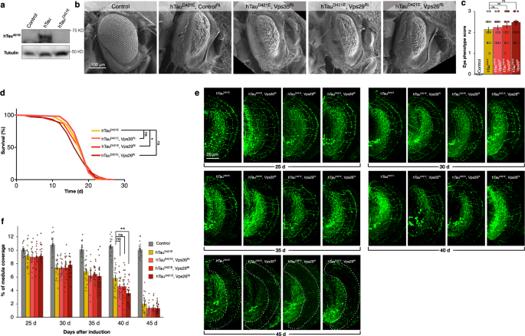Fig. 4: Abolishing Tau truncation abrogates enhancement of toxicity by retromer inhibition. aProtein analyses of Tau421Dtruncated isoform levels in control [GMR-Gal4, UAS-mCD8GFP], hTau expressing [GMR-Gal4, UAS-hTau] and hTauD421Emutant expressing [GMR-Gal4, UAS-hTauD421E] animals.bEye morphology of control [GMR-Gal4, UAS-mCD8GFP], hTauD421Eexpressing [GMR-Gal4, UAS-hTauD421E, UAS-GFPRi], and hTauD421E[GMR-Gal4, UAS- hTauD421E] expression plus inhibition of retromer components [UAS-Vps35Rior UAS-Vps29Rior UAS-Vps26Ri] animals.cEye disruption scores for control [GMR-Gal4, UAS-mCD8GFP], hTauD421Eexpressing [GMR-Gal4, UAS-hTauD421E, UAS-GFPRi] and hTauD421E[GMR-Gal4, UAS- hTauD421E] expression plus inhibition of retromer components [UAS-Vps35Rior UAS-Vps29Rior UAS-Vps26Ri] animals. Data are presented as mean values +/− SEM.dSurvival analyses of hTauD421Eexpressing [dTau-Gal4, UAS-hTauD421E, UAS-CherryRi,tubulin-Gal80ts] and hTauD421E[dTau-Gal4, UAS-hTauD421E,tubulin-Gal80ts] expression together with retromer inhibition [UAS-Vps35Rior UAS-Vps29Rior UAS-Vps26Ri] adults.eExample DC neuron medulla axons in hTauD421Eexpressing alone [ato-Gal4, UAS-hTauD421E, UAS-mCherry, UAS-mCD8GFP,tubulin-Gal80ts], and hTauD421Eexpressing [ato-Gal4, UAS-hTauD421E, UAS-mCherry,tubulin-Gal80ts] together with retromer inhibition [UAS-Vps35Rior UAS-Vps29Rior UAS-Vps26Ri], from 25 to 45 days after onset of transgene expression. Gaps in the axonal structures are indicated with arrowheads. In brains with <4% axons, the medulla is outlined with broken lines.fQuantification of medulla area occupied by DC neuron axons in control [ato-Gal4, UAS-mCherry, UAS-mCD8GFP,tubulin-Gal80ts], hTauD421Eexpressing alone [ato-Gal4, UAS-hTauD421E, UAS-mCherry, UAS-mCD8GFP,tubulin-Gal80ts], and hTauD421Eexpressing [ato-Gal4, UAS-hTauD421E, UAS-mCherry,tubulin-Gal80ts] together with retromer inhibition [UAS-Vps35Rior UAS-Vps29Rior UAS-Vps26Ri]. Data are presented as mean values +/− SEM. Kruskal–Wallis test,p= 0.3272 for eye disruption scores across all genotypes with multiple comparisons between hTauD421E(n= 33) and hTauD421Eplus Vps35Ri(n= 30) (Dunnett’s testp= 0.1716), hTauD421Eand hTauD421Eplus Vps29Ri(n= 31) (Dunnett’s testp= 0.5443), and hTauD421Eand hTauD421Eplus Vps26Ri(n= 29) (Dunnett’s testp= 0.9899),n= 32 for control (c). Mantel-Cox test,p= 0.2508 for survival analysis of hTauD421E(n= 248) vs. hTauD421Eplus Vps35Ri(n= 218), *p= 0.0105 for hTauD421Evs. hTauD421Eplus Vps29Ri(n= 233), andp= 0.0988 for hTauD421Eand hTauD421Eplus Vps26Ri(n= 260) (d). Kruskal–Wallis test,p= 0.9847 (f, 25 days post induction) with multiple comparisons between hTauD421E(n= 20) and hTauD421Eplus Vps35Ri(n= 19) (Dunnett’s testp= 0.9873), hTauD421Eand hTauD421Eplus Vps29Ri(n= 20) (Dunnett’s testp= 0.9557), and hTauD421Eand hTauD421Eplus Vps26Ri(n= 18) (Dunnett’s testp= 0.9999),n= 18 for control. Kruskal–Wallis test,p= 0.9552 (f, 30 days post induction), with multiple comparisons between hTauD421E(n= 19) and hTauD421Eplus Vps35Ri(n= 16) (Dunnett’s testp= 0.9991), hTauD421Eand hTauD421Eplus Vps29Ri(n= 20) (Dunnett’s testp= 0.9999), and hTauD421Eplus Vps26Ri(n= 18) (Dunnett’s testp= 0.9714),n= 20 for control. Kruskal-Wallis test,p= 0.4127 (f, 35 days post induction), with multiple comparisons between hTauD421E(n= 18) and hTauD421Eplus Vps35Ri(n= 16) (Dunnett’s testp= 0.5464), hTauD421Eand hTauD421Eplus Vps29Ri(n= 20) (Dunnett’s testp= 0.8007), and hTauD421Eplus Vps26Ri(n= 19) (Dunnett’s testp= 0.4417),n= 17 for control. Kruskal–Wallis test, *p= 0.0127 (f, 40 days post induction), with multiple comparisons between hTauD421E(n= 19) and hTauD421Eplus Vps35Ri(n= 20) (Dunnett’s testp= 0.108), hTauD421Eand hTauD421Eplus Vps29Ri(n= 19) (Dunnett’s testp= 0.111), and hTauD421Eplus Vps26Ri(n= 19) (Dunnett’s test **p= 0.0013),n= 18 for control. Kruskal–Wallis test,p= 0.4553 (f, 45 days post induction), with multiple comparisons between hTauD421E(n= 20) and hTauD421Eplus Vps35Ri(n= 11) (Dunnett’s testp= 0.2311), hTauD421Eand hTauD421Eplus Vps29Ri(n= 13) (Dunnett’s testp= 0.3127), and hTauD421Eplus Vps26Ri(n= 20) (Dunnett’s test **p= 0.1683),n= 19 for control. n indicates independent biological replicates. Source data are provided as a Source Data file. Drosophila phenotypic analysis Eye phenotypes were imaged, using Leica DFC 3000 G and scored blind to genotype using a modified version of published criteria [32] as described in Supplementary Fig. 1 and in supplementary methods. Preparation of scanning electron micrographs are described in supplemental methods and were imaged using a Zeiss Merlin Scanning Electron Microscope. To label DC neuron axons and express transgenes we generated a line that combined ato -Gal4 [38] with UAS-mCherry [6X] [101] . The expression of transgenes by this line during development was inhibited by combining it with temperature-sensitive Gal80 (Tub-Gal80 ts ) [34] which suppresses Gal4-dependent expression at 18 °C but allows expression at 29 °C. Animals of the desired genotype were grown at 18 °C until 3 days after eclosion and then transferred to 29 °C. Under these expression conditions, control animals lived to a maximal age of 50 days. Entire adult brains were stained and imaged using a Zeiss LSM700. Quantification of DC neuron medulla axon coverage was performed blind to genotype using the threshold tool in ImageJ [102] . Briefly, medulla areas were cropped from Z projections of brain images. Pixel intensity was then set such that axons were above threshold. The percentage of medulla area occupied by axons was then measured. Brain dissection, staining procedures, and antibodies employed are described in supplementary methods. Protein measurements Protein measurements were performed using adult head lysates and imaged using an Amersham Imager 680 or Vilber Lourmat Fusion FX. Densitometric analyses of western blots were quantitated using the Gels tool of ImageJ. The following antibodies were used: mouse anti-cleaved-Tau (Asp421) clone C3 (Millipore; 36-017) 1:1000, rabbit anti-TauC (1:20,000), rabbit anti-PHF-1 (Sigma) 1:2000, monoclonal anti-phospho-Tau (Ser202, Thr205) (AT8) (Thermo Fisher) 1:2000, monoclonal anti-phospho-Tau (Thr212, Ser214) (AT100) (Thermo Fisher) 1:2000, monoclonal anti-Spectrin (DSHB) 1:1000, monoclonal anti-alpha tubulin (Sigma) 1:2000, mouse anti-HA (Covance) 1:1000, guinea pig anti-Vps26 (gift from Hugo Bellen) (1:4000), HRP anti-mouse (Jackson Immunoresearch) (1:20,000), HRP anti-rabbit (Jackson ImmunoResearch) (1:20,000), HRP anti-guinea pig (1:20,000). Additional details on head lysate preparation, immunoprecipitation, and antibody staining procedures are described in supplemental methods. Mammalian cell culture Immortalized CN1.4 mouse cortical neurons that stably express inducible forms of hTau [2N4R] were described previously [50] . To inhibit retromer in these lines we used lentivirus expression of murine VPS26A, VPS29 or VPS35 shRNA or a scrambled shRNA control. Cell culture conditions, lentivirus preparation, transduction, and protein measurement procedures are described in supplemental methods. Statistics Prior to performing statistical analyses, the distribution of data was checked, for all datasets, using a Shapiro-Wilk normality test. In the event of non-normal distribution, even for one group in a large dataset (for example, a timepoint in axon degeneration dataset), a non-parametric test was chosen. The following tests were employed—for Drosophila eye phenotypes: non-parametric Mann–Whitney U test or Kruskal–Wallis test with Dunnett’s multiple comparison test; for synapse and axon degeneration: Unpaired two-tailed t -test, one-way ANOVA or Kruskal–Wallis test along with Dunnett’s multiple comparison test; for protein levels analysis: Unpaired two-tailed t -test or one-way ANOVA along with Tukey’s multiple comparison test. For multiple comparisons, adjusted p values are reported. Statistical analyses were performed using GraphPad PRISM 7.0a. Ethical approval Studies using Drosophila melanogaster are not subject to institutional ethical approval however all experiments complied with relevant guidelines. 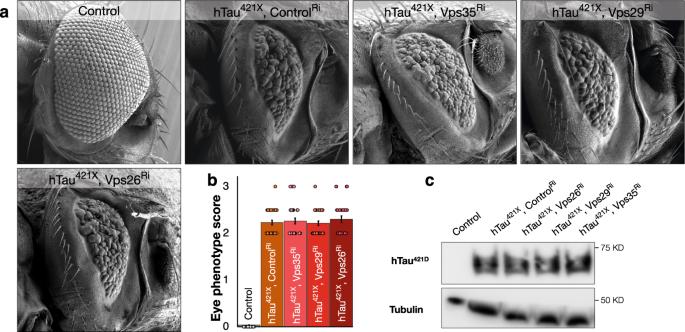Fig. 5: The toxicity of extant truncated Tau is not enhanced by retromer depletion. aEyes from control [GMR-Gal4, UAS-mCD8GFP], hTau421Xexpressing [GMR-Gal4, UAS-hTau421X, UAS-GFPRi] animals, and hTau421X[GMR-Gal4, UAS-hTau421X] expressing together with retromer inhibition [UAS-Vps35Rior UAS-Vps29Rior UAS-Vps26Ri] animals.bEye disruption scores for control [GMR-Gal4, UAS-mCD8GFP], hTau421Xexpressing [GMR-Gal4, UAS-hTau421X, UAS-GFPRi] animals, and hTau421X[GMR-Gal4, UAS-hTau421X] expressing together with retromer inhibition [UAS-Vps35Rior UAS-Vps29Rior UAS-Vps26Ri] animals. Data are presented as mean values +/− SEM.cTruncated Tau (hTau421D) levels from head lysates of control [GMR-Gal4, UAS-mCD8GFP], hTau421Xexpressing [GMR-Gal4, UAS-hTau421X, UAS-GFPRi], and hTau421Xexpressing [GMR-Gal4, UAS-hTau421X] together with retromer inhibition [UAS-Vps35Rior UAS-Vps29Rior UAS-Vps26Ri] animals. Kruskal–Wallis test,p= 0.8297 for eye disruption scores across all genotypes with multiple comparisons between hTau421X(n= 30) and hTau421Xplus Vps35Ri(n= 30) (Dunnett’s testp= 0.8779), hTau421Xand hTau421Xplus Vps29Ri(n= 32) (Dunnett’s testp= 0.9999), and hTau421Xand hTau421Xplus Vps26Ri(n= 31) (Dunnett’s testp= 0.564).nindicates independent biological replicates. Source data are provided as a Source Data file. 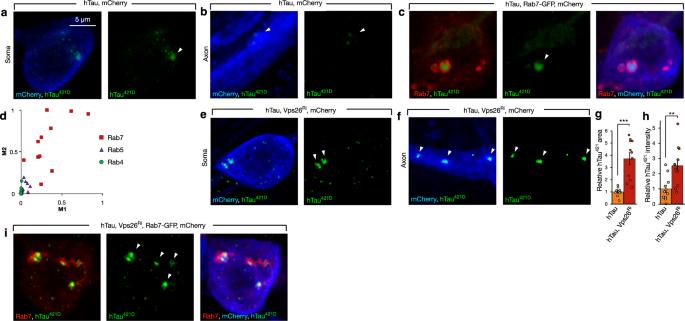Fig. 6: Reduction of Retromer leads to accumulation of truncated Tau in late endosomes. a,bLeft panel: Soma and axons of dHB9 neurons expressing hTau and mCherry (blue) [dHB9-Gal4, UAS-hTau, UAS-mCherry, UAS-mCD8GFP]. hTau421D(green) accumulates in discrete subcellular compartments. Right panels: hTau421Daccumulations labeled by arrowheads.cLeft panel: hTau421D(green) encapsulated in late endosomal compartments labeled with Rab7-GFP (red) in the soma of dHB9 expressing hTau neurons [dHB9-Gal4, UAS-hTau, UAS-Rab7-GFP, UAS-mCherry]. Middle panel: hTau421Daccumulations labeled by arrowheads. Right panel: Rab7-GFP (red), hTau421D(green) and mCherry (blue).dMander’s analyses of the spatial relationship of hTau421Dwith endosomes labeled by either Rab4-GFP (n= 12), Rab5-GFP (n= 12) or Rab7-GFP (n= 11). M1 is the fraction of each Rab protein overlapping with Tau421D, while M2 is the fraction of Tau421Dsignal overlapping with each Rab protein signal.e,fLeft panels: hTau421Daccumulations (green) in the soma (e) and axons (f) of hHB9 neurons (mCherry, blue) expressing hTau together with retromer inhibition [dHB9-Gal4, UAS-hTau, UAS-Vps26Ri, UAS-mCherry]. Right panels: hTau421Daccumulations labeled by arrowheads.gRelative area of hTau421Daccumulations normalized to neuronal area in dHB9 neurons expressing hTau [dHB9-Gal4, UAS-hTau, UAS-mCherry, UAS-mCD8GFP] and when retromer is inhibited [dHB9-Gal4, UAS-hTau, UAS-mCherry, UAS-Vps26Ri]. Data are presented as mean values +/− SEM.hIntensity of hTau421Daccumulations normalized to mCherry in dHB9 neurons expressing hTau [dHB9-Gal4, UAS-hTau, UAS-mCherry, UAS-mCD8GFP] and when retromer is inhibited [dHB9-Gal4, UAS-hTau, UAS-mCherry, UAS-Vps26Ri]. Data are presented as mean values +/− SEM.iLeft panel: hTau421D(green) encapsulated in late endosomal compartments labeled with Rab7-GFP (red) in the soma ofdHB9expressing hTau neurons when retromer is inhibited [dHB9-Gal4, UAS-hTau, UAS-Rab7-GFP, UAS-mCherry, UAS-Vps26Ri]. Middle panel: hTau421Daccumulations labeled by arrowheads. Right panel: Rab7-GFP (red), hTau421D(green) and mCherry (blue). Unpaired two-tailedt-test,***p< 0.001, hTau vs. hTau plus Vps26Ri(n= 11 neurons examined over three independent experiments) (g). Unpaired two-tailedt-test,**p= 0.0039, hTau vs. hTau plus Vps26Ri(n= 11 neurons examined over three independent experiments) (h). n indicates independent biological replicates. Source data are provided as a Source Data file. 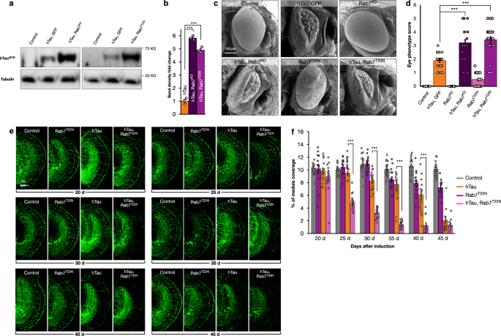Fig. 7: Rab7 inhibition increases Tau truncation. ahTau421Dprotein level analyses from head lysates of controls [GMR-Gal4, UAS-mCD8GFP], hTau expressing [GMR-Gal4, UAS-hTau, UAS-DeGradFP] and hTau expressing together with Rab7 knock-down (Rab7KD) [GMR-Gal4, UAS-hTau, Rab7EYFP/ΔRab7, UAS-DeGradFP] or Rab7T22Nexpression [GMR-Gal4, UAS-hTau, UAS-Rab7T22N] animals.bQuantification of hTau421Dprotein levels from head lysates of controls [GMR-Gal4, UAS-mCD8GFP], hTau expressing [GMR-Gal4, UAS-hTau, UAS-DeGradFP] and hTau expressing together with Rab7 knock-down (Rab7KD) [GMR-Gal4, UAS-hTau, Rab7EYFP/ΔRab7, UAS-DeGradFP] or Rab7T22Nexpression [GMR-Gal4, UAS-hTau, UAS-Rab7T22N] animals. Data are presented as mean values +/− SEM.cEyes from control [GMR-Gal4, UAS-mCD8GFP], hTau expressing [GMR-Gal4, UAS-hTau, UAS-mCD8GFP], Rab7 knockdown alone (Rab7KD) [GMR-Gal4, Rab7EYFP/ΔRab7, UAS-DeGradFP], hTau expressing with Rab7KD[GMR-Gal4, UAS-hTau, Rab7EYFP/ΔRab7, UAS-DeGradFP], Rab7 inhibition (Rab7T22N) alone [GMR-Gal4, UAS-Rab7T22N, UAS-mCD8GFP], and hTau expression together with Rab7T22N[GMR-Gal4, UAS-hTau, UAS-Rab7T22N] animals.dEye disruption scores from control [GMR-Gal4, UAS-mCD8GFP], hTau expressing [GMR-Gal4, UAS-hTau, UAS-DeGradFP], Rab7KD[GMR-Gal4, Rab7EYFP/ΔRab7, UAS-DeGradFP], hTau expressing with Rab7KD[GMR-Gal4, UAS-hTau, Rab7EYFP/ΔRab7, UAS-DeGradFP], Rab7T22N[GMR-Gal4, UAS-Rab7T22N, UAS-mCD8GFP], and hTau expression together with Rab7T22N[GMR-Gal4, UAS-hTau, UAS-Rab7T22N] animals. Data are presented as mean values +/− SEM.eExample DC neuron medulla axons from control [ato-Gal4, UAS-mCherry, UAS-mCD8GFP,tubulin-Gal80ts], Rab7T22Nexpression alone [ato-Gal4, UAS-Rab7T22N, UAS-mCherry,tubulin-Gal80ts], hTau expression alone [ato-Gal4, UAS-hTau, UAS-mCherry, UAS-mCD8GFP,tubulin-Gal80ts], and hTau expression together with Rab7 inhibition [ato-Gal4, UAS-hTau, UAS-Rab7T22N, UAS-mCherry,tubulin-Gal80ts] animals from 20 to 45 days after onset of transgene expression. Gaps in axonal structure induced by hTau expression are indicated with arrowheads, when < 4% axons are present, the medulla is outlined with dashed lines.fQuantification of medulla area occupied by DC neuron from control [ato-Gal4, UAS-mCherry, UAS-mCD8GFP,tubulin-Gal80ts], Rab7T22Nexpression alone [ato-Gal4, UAS-Rab7T22N, UAS-mCherry,tubulin-Gal80ts], hTau expression alone [ato-Gal4, UAS-hTau, UAS-mCherry, UAS-mCD8GFP,tubulin-Gal80ts], and hTau expression together with Rab7 inhibition [ato-Gal4, UAS-hTau, UAS-Rab7T22N, UAS-mCherry,tubulin-Gal80ts] 20–45 days after onset of transgene expression. Data are presented as mean values +/− SEM. Unpaired two-tailedt-test,p< 0.001, (b, hTau421D) for hTau (n= 3) vs. hTau plus Rab7KD(n= 3), andp< 0.001 for hTau (n= 3) vs. hTau plus Rab7T22N(n= 3). Kruskal–Wallis test, ***p< 0.001 for eye disruption scores across all genotypes with multiple comparisons between hTau (n= 26) and hTau plus Rab7KD(n= 26) (Dunnett’s test ***p< 0.001), and hTau and hTau plus Rab7T22N(n= 28).n= 32 for control,n= 30 for Rab7KD, andn= 28 for Rab7T22N(d). Mann–Whitney test,p= 0.2928 for hTau (n= 15) vs. hTau plus Rab7T22N(n= 18) (f, 20 days post induction,n= 15 for control andn= 16 for Rab7T22N). Mann–Whitney test, ***p< 0.001 for hTau (n= 16) vs. hTau plus Rab7T22N(n= 15) (f, 25 days post induction,n= 18 for control andn= 17 for Rab7T22N). Mann–Whitney test, ***p< 0.001 for hTau (n= 20) vs. hTau plus Rab7T22N(n= 17) (f, 30 days post induction,n= 20 for control andn= 15 for Rab7T22N). Mann–Whitney test, ***p< 0.001 for hTau (n= 20) vs. hTau plus Rab7T22N(n= 18) (f, 35 days post induction,n= 17 for control andn= 15 for Rab7T22N). Mann–Whitney test, ***p< 0.001 for hTau (n= 20) vs. hTau plus Rab7T22N(n= 12) (f, 40 days post induction,n= 18 for control andn= 14 for Rab7T22N). Mann–Whitney test,p= 0.7132 for hTau (n= 20) vs. hTau plus Rab7T22N(n= 10) (f, 45 days post induction,n= 19 for control andn= 14 for Rab7T22N).nindicates independent biological replicates. Source data are provided as a Source Data file. 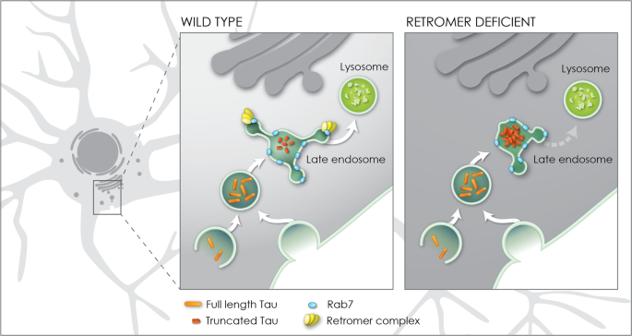Fig. 8: Model for enhancement of Tau toxicity and truncation by retromer depletion. In wildtype neurons full length Tau (orange) enters the endosomal network and is efficiently trafficked through the late endosome to the lysosome enabled by the interaction of the retromer complex (yellow) with the late endosome protein Rab7 (blue). When retromer or Rab7 activity is reduced, endosomal-lysosomal flux is retarded, exposing Tau to endosomal resident caspase activity which results in Tau truncation (red) and accumulation in the late endosome. Truncation of Tau enhances its neurotoxicity. Reporting summary Further information on research design is available in the Nature Research Reporting Summary linked to this article.